Transcriptional network involving ERG and AR orchestrates Distal-less homeobox-1 mediated prostate cancer progression Distal-less homeobox-1 (DLX1) is a well-established non-invasive biomarker for prostate cancer (PCa) diagnosis, however, its mechanistic underpinnings in disease pathobiology are not known. Here, we reveal the oncogenic role of DLX1 and show that abrogating its function leads to reduced tumorigenesis and metastases. We observed that ~60% of advanced-stage and metastatic patients display higher DLX1 levels. Moreover, ~96% of TMPRSS2-ERG fusion-positive and ~70% of androgen receptor (AR)-positive patients show elevated DLX1 , associated with aggressive disease and poor survival. Mechanistically, ERG coordinates with enhancer-bound AR and FOXA1 to drive transcriptional upregulation of DLX1 in ERG-positive background. However, in ERG-negative context, AR/AR-V7 and FOXA1 suffice to upregulate DLX1 . Notably, inhibiting ERG/AR-mediated DLX1 transcription using BET inhibitor (BETi) or/and anti-androgen drugs reduce its expression and downstream oncogenic effects. Conclusively, this study establishes DLX1 as a direct-target of ERG/AR with an oncogenic role and demonstrates the clinical significance of BETi and anti-androgens for DLX1-positive patients. Recurrent gene rearrangements involving the androgen-regulated transmembrane protease serine 2 ( TMPRSS2) and ETS transcription factor, v-ets erythroblastosis virus E26 oncogene homolog ( ERG) occur in ~50% of prostate cancer (PCa) patients [1] . Aberrant overexpression of ERG controls a transcriptional network linked to PCa development [2] , [3] , increased metastatic potential, and associate with poor clinical outcome [4] . In TMPRSS2-ERG fusion-positive PCa, ERG recruitment onto the SOX9 promoter opens up cryptic androgen receptor (AR) binding sites on the SOX9 enhancer thereby regulating its expression, while the loss of SOX9 results in reduced ERG-mediated oncogenicity [5] . Nonetheless, other critical partners that govern ERG-mediated oncogenesis remain largely unexplored. Considering the critical role of AR signaling in the development and progression of PCa, inhibitors targeting androgen synthesis (abiraterone acetate) and AR antagonists (bicalutamide, enzalutamide) are used in the first line of treatment termed androgen deprivation therapy (ADT), often administered to advanced stage PCa patients [6] . Although, prolonged administration of ADT results in an inevitable cancer relapse due to the selection pressure of drugs, eventually progressing to aggressive castration-resistant prostate cancer (CRPC) stage [6] . Recent drugs such as apalutamide and darolutamide prolong the metastatic-free survival of CRPC patients [7] . In addition, the Food and Drug Administration (FDA) has also approved the use of apalutamide for non-metastatic, castration-sensitive patients [8] . Mounting evidence suggests sustained AR activity in CRPC, owing to numerous mechanisms including AR amplification, gene mutations, intra-tumoral androgen synthesis, and expression of constitutively active AR splice variants (AR-Vs) [6] . Moreover, patients treated with enzalutamide and abiraterone showed increased levels of AR-V7 in the circulating tumor cells, and shorter time to biochemical relapse compared to AR-V7 negative cases [9] . Unlike full-length AR (AR-FL), the splice variant AR-V7 functions in a ligand-independent manner and remains constitutively active driving androgen-independent growth and disease progression [10] . Interestingly, a recent study showed a distinct AR-V7 cistrome that governs cell-context-dependent gene expression [11] . Recent studies revealed the clinical significance of bromodomain and extra-terminal (BET) domain proteins, which are known transcriptional coactivators of tumor-promoting genes such as AR and are considered as a potential therapeutic target for CRPC treatment [12] , [13] . The Distal-less homeobox (DLX) genes belong to the homeobox-containing family of transcription factors (TFs), which are structural homologs of Drosophila Distal-less (Dll). DLX1 being a member of the DLX family plays an essential role in the development of craniofacial features, jaw, and GABAergic (gamma-aminobutyric acid) interneuron [14] . Deregulation of homeobox genes has been linked to several human malignancies including prostate [15] . In hematopoietic cells, DLX1 impedes downstream TGF-β-mediated signaling pathways by interacting with Smad4 [16] . In PCa, DLX1 is known to functionally interact with β-catenin and regulate downstream β-catenin/TCF4 signaling pathway [17] . Furthermore, DLX1 has been validated as a PCa biomarker across clinically independent cancer cohorts, wherein DLX1 and HOXC6 accurately predict high-grade disease [18] . However, the underlying regulatory mechanism that drives DLX1 upregulation and its functional role in PCa progression remain poorly understood. Here, we uncover the molecular mechanisms underlying the upregulation of DLX1 in PCa and reveal oncogenic functions associated with it. Our data identify DLX1-mediated downstream biological processes that operate in PCa tumorigenesis and show its oncogenic role in disease progression and metastasis. We also demonstrate the role of ERG, AR, and FOXA1 as key transcriptional regulators involved in DLX1 overexpression in PCa. Lastly, we show that disrupting ERG/AR transcriptional circuitry with BET inhibitor (BETi) or in combination with anti-androgen could attenuate DLX1-mediated tumorigenesis. Collectively, this study highlights the importance of DLX1 as an effective therapeutic target in PCa patients irrespective of TMPRSS2-ERG fusion status. DLX1 imparts oncogenic properties and promotes PCa progression To study the association between increased DLX1 levels and PCa progression, we analyzed RNA-sequencing (RNA-Seq) data using publicly available clinical genomics data repository viz. The Cancer Genome Atlas Prostate Adenocarcinoma (TCGA-PRAD) dataset. Interestingly, higher expression of DLX1 was observed in patients with primary PCa compared to matched normal tissue (Fig. 1a ). Similarly in other clinical genomics datasets (GSE35988 [19] and GSE80609 [20] ) an increased expression of DLX1 transcript was observed in advanced stage aggressive cancers compared to benign (Fig. 1b and Supplementary Fig. 1a ). In agreement with this, patients with higher DLX1 expression ( DLX1 Hi ) experienced poor survival probability compared to those with lower DLX1 expression ( DLX1 Lo ) (Fig. 1c ). Likewise, elevated DLX1 levels were observed in PCa cell lines (22RV1, VCaP, and PC3) that represent CRPC compared to LNCaP cells, an androgen-responsive, and RWPE1, a benign and immortalized prostate epithelial cell line (Supplementary Fig. 1b ). Also, the read coverage of DLX1 transcript from the RNA-Seq data of RWPE1 [21] , 22RV1 [22] , and VCaP [22] cell lines showed similar trends (Fig. 1d ). To understand the functional significance of DLX1 in PCa, we ectopically overexpressed DLX1 in RWPE1 cells and confirmed its overexpression both at transcript and protein levels (Supplementary Fig. 1c ). Interestingly, a significant increase in cell proliferation in RWPE1-DLX1 cells compared to control was observed (Fig. 1e ). Similarly, DLX1 overexpression markedly increased foci forming ability and migratory properties of RWPE1 cells (Fig. 1f, g ). In contrast, to understand the functional role of DLX1 using a loss-of-function model, CRISPR/Cas9 mediated gene knockout of DLX1 was performed in 22RV1 cells (Supplementary Fig. 1d ), and DLX1 knockout (KO) was confirmed by genomic amplification of the CRISPR/Cas9 target gene sequence (Supplementary Fig. 1e ). Three independent DLX1 -KO clones, namely 22RV1- DLX1 -KO (C-1, C-2, and C-3) showing loss of DLX1 expression both at transcript and protein levels (Supplementary Fig. 1f ) were selected to determine any phenotypic changes in these genetically engineered lines. Notably, a marked reduction in proliferation rates of 22RV1- DLX1- KO cells was observed compared to control (Fig. 1h ). Similarly, a significant reduction (~60%) in the cell migratory and foci forming properties was observed in 22RV1- DLX1 -KO cells (Fig. 1i and Supplementary Fig. 1g ). We also observed a ~4–5-fold decrease in the anchorage-independent growth of 22RV1- DLX1 -KO cells compared to control (Fig. 1j ). Fig. 1: High DLX1 expression associates with poor prostate cancer prognosis and promotes disease progression. a Dot plot showing DLX1 expression in PCa patients ( n = 498) and matched normal ( n = 52) in TCGA-PRAD RNA-Seq dataset, data represents log2 (norm_count+1), center depicts mean ± (standard deviation) SD ( P < 0.0001). b Dot plot of DLX1 expression using microarray profiling data (GSE35988) comprising benign ( n = 28), localized ( n = 59), and mCRPC ( n = 35) patient specimens, data represents log2 (norm_mRNA), center depicts mean ± SD ( P < 0.0001). c Kaplan–Meier plot showing survival probability in TCGA-PRAD ( n = 498) dataset categorized in high DLX1 ( DLX1 Hi ) and low DLX1 ( DLX1 Lo ) expression. d RNA-Seq data showing DLX1 transcript read counts in publicly available datasets (GSE128399 and GSE118206). e Cell proliferation assay using isogenic RWPE1 cells overexpressing DLX1 at indicated time-points ( P < 0.0001). f Foci formation assay using same cells as e ( P < 0.0001). g Boyden Chamber Matrigel migration assay using same cells as e ( P < 0.0001). Representative images for panels f (scale bar 500 µm) and g (scale bar 100 µm) are shown as inset. h Cell proliferation assay using 22RV1- DLX1 -KO (C-1, C-2, and C-3 are independent clones) and control cells at indicated time-points ( P < 0.0001). i Boyden Chamber Matrigel migration assay using same cells as h ( P < 0.0001). j Anchorage-independent soft agar assay using same cells as h ( P < 0.0001). Representative images for panels i and j are shown as inset (scale bar 100 µm). k DAVID analysis showing upregulated (right) and downregulated (left) biological processes in 22RV1- DLX1 -KO against control cells. Bars represent the −log 10 ( P -value) and the frequency polygon (black line) denotes number of genes. l Same as k , except gene set enrichment analysis (GSEA) plots representing deregulated pathways. m Heatmap displaying downregulated genes involved in cancer stemness and EMT in 22RV1- DLX1 -KO cells compared to control. Data shown from three biologically independent samples ( n = 3). Data represent mean ± SEM unless specified. For panels, a Unpaired Student’s two-tailed t -test was applied; b One-way ANOVA with Dunnett’s multiple comparison test was applied; e Two-way ANOVA Sidak’s multiple comparison test; f , g Unpaired two-tailed Welch’s t -test; h Two-way ANOVA, Dunnett’s multiple comparisons test; i , j One-way ANOVA, Dunnett’s multiple comparisons test was applied. Source data are provided as a Source Data file. Full size image To delineate the biological pathways orchestrated by DLX1 in PCa, we performed a microarray-based global gene expression profiling of 22RV1- DLX1 -KO and 22RV1-SCR cells. Database for Annotation, Visualization and Integrated Discovery (DAVID, https://david.ncifcrf.gov/ ) bioinformatics analysis on the differentially expressed genes (log 2 fold-change >0.6 or <−0.6, 90% confidence interval) revealed significantly up- and downregulated biological processes engaged by DLX1 (Supplementary Data 1 ). As anticipated, genes involved in proliferation and migration of cells, and stem-cell population maintenance were negatively enriched in 22RV1- DLX1 -KO cells, while genes associated with cell cycle regulation and antigen processing and presentation were upregulated (Fig. 1k ). Subsequent gene set enrichment analysis (GSEA) showed enrichment of genes involved in the apoptotic pathway in DLX1 -KO cells, whereas gene sets involved in epithelial-to-mesenchymal transition (EMT), cancer stemness, active Akt, and Wnt signaling were enriched in the control cells (Fig. 1l, m ). To further explore the oncogenic role of DLX1 in aggressive PCa, we analyzed RNA-Seq data (GSE78913) [23] for the transient knockdown of DLX1 in LNCaP derivative osteotropic cell line C4-2B, and as speculated DLX1 was found to be one of the top five downregulated genes as depicted in the volcano plot (Supplementary Fig. 1h ). In addition, GSEA and pathway analysis of the differentially expressed genes showed deregulation of important pathways associated with cancer, such as upregulation of apoptosis and cell cycle arrest (Supplementary Fig. 1i, j ). Further, functional characterization of differentially expressed genes in the 22RV1- DLX1 -KO cells by an overlapping network-based analysis revealed significant ( P < 0.005, FDR < 0.1) downregulation of EMT, cell cycle and DNA damage pathways (Supplementary Fig. 2 ). Taken together, our findings implicate the critical role of DLX1 in imparting oncogenic properties to prostate cells. DLX1 elicits biological processes involved in cancer progression To investigate the underlying mechanism involved in oncogenic properties imparted by DLX1, we examined the expression of genes involved in EMT at the transcript and protein level. Reduced expression of two archetypal markers of the mesenchymal phenotype, namely Vimentin and Snail, with increased E-cadherin expression, an epithelial marker in DLX1 -KO cells was observed (Fig. 2a, b ). Conversely, increased vimentin expression was observed in DLX1 overexpressing RWPE1 cells (Supplementary Fig. 3a ). Consistent with the GSEA data, an increased apoptosis marked by Caspase 3 activation and cleaved poly-(ADP-ribose) polymerase (PARP) in DLX1 -KO cells along with decrease in the levels of anti-apoptotic Bcl-xL was observed (Fig. 2c ). Concurrently, increased expression of late apoptotic markers was noted as shown by a rise in the number of Annexin-V and 7-AAD (7-amino-actinomycin D) stained 22RV1- DLX1 -KO cells (Fig. 2d ). In line with this, DLX1 silencing in VCaP cells also augment apoptosis as shown by an increase in the number of Annexin-V and 7-AAD positive cells (Fig. 2d and Supplementary Fig. 3b ). Next, our flow-cytometry-based cell cycle analysis revealed an increase in the percentage of cells arrested in the S-phase with a concomitant decrease in the G2/M phase cells in DLX1 -KO compared to control (Fig. 2e ). Similarly, small interfering RNA (siRNA)-mediated transient knockdown of DLX1 in VCaP cells resulted in cell cycle arrest (Fig. 2e ). Although, the cell cycle arrest in transiently DLX1 -silenced VCaP cells was not as robust as observed in CRISPR-based DLX1 knockout in 22RV1. Furthermore, an increase in the phospho-Akt (pAkt) levels was observed in RWPE1-DLX1 cells (Supplementary Fig. 3a ), indicating the critical role of DLX1 in regulating cancer cell survival and proliferation. Fig. 2: Genetic ablation of DLX1 inhibits oncogenic properties. a Q-PCR data showing expression of EMT markers in 22RV1- DLX1 -KO and control SCR cells. b Immunoblots showing vimentin and E-cadherin using same cells as a . β-actin was used as loading control. c Same as b except for cleaved PARP, cleaved Caspase-3 and Bcl-xL. d Flow cytometry-based apoptosis assay using 22RV1- DLX1 -KO and control cells (top panel) and DLX1 -silenced VCaP cells (bottom panel). e Flow cytometry data for cell cycle distribution using same cells as in d . f Q-PCR data for stem cell markers using same cells as d . g Flow cytometry data depicting ABCG2 (top panel) and CD44 (bottom panel) expression in DLX1 overexpressing RWPE1 cells, 22RV1- DLX1 -KO, and DLX1 -silenced VCaP cells. h Fluorescence intensity of catalyzed ALDH substrate in 22RV1- DLX1 -KO and control cells. Marked windows show ALDH1 + percent cell population. i Same as h , except for DLX1 silenced VCaP cells. j Q-PCR data showing expression of target genes in 22RV1- DLX1 -KO and control cells( P < 0.0001). k Schema showing the chromosomal location of DLX1 binding motif (DBM1/2) at the ALDLH1A1 (top) and HNF1A (bottom) promoters. l ChIP-qPCR data of DLX1 (top panel) and H3K9Ac (bottom panel) on ALDH1A1 in 22RV1- DLX1 -KO and SCR control cells ( P < 0.0001). m Same as in l except for the HNF1A promoter. Data shown from three biologically independent samples ( n = 3). Data represent mean ± SEM. For panels, a , f , and j Two-way ANOVA, Dunnett’s multiple comparison test; l , m Two-way ANOVA Turkey’s multiple comparison test was applied. Source data are provided as a Source Data file. Full size image In agreement with the microarray data, DLX1 -KO cells exhibit decreased expression of established stem cell markers such as POU5F1 (Oct-4), ABCG2 , CD117 (c-KIT), and SOX2 (Fig. 2f ). Next, we examined the cell surface expression of two well-known stem cell markers, ABCG2 and CD44 in 22RV1- DLX1 -KO, DLX1 -silenced VCaP, and RWPE1-DLX1 cells. Interestingly, a marked reduction in the expression of ABCG2 (~30–60%) and CD44 (~50–80%) was observed in 22RV1- DLX1 -KO and DLX1- silenced VCaP cells, while a robust increase in these markers was noted in RWPE1-DLX1 cells (Fig. 2g ). Since increased aldehyde dehydrogenase 1A1 (ALDH1A1) activity is often associated with cancer stem cell phenotype [24] , we performed ALDH activity assay using RWPE1-DLX1 cells that showed a significant increase in ALDH activity (Supplementary Fig. 3c ). Conversely, 22RV1- DLX1 -KO and DLX1- silenced VCaP cells showed reduction in the ALDH activity (Fig. 2h, i ), indicating a plausible function of DLX1 in promoting cancer stemness. Furthermore, to confirm the oncogenic role of DLX1 in enzalutamide-resistant PCa, we silenced DLX1 in LNCaP derivative enzalutamide-resistant 42D cells (42D ENZ R ) (Supplementary Fig. 3d ). Interestingly, DLX1 silencing in 42D ENZ R cells resulted in S-phase cell cycle arrest and increased expression of apoptotic markers (Supplementary Fig. 3e, f ). Furthermore, DLX1 silencing was marked with reduced ALDH activity in 42D ENZ R cells (Supplementary Fig. 3g ). Together, these data highlight the possible role of DLX1 in promoting cancer stemness, EMT, and proliferation in PCa. To explore the DLX1 target genes which are involved in tumorigenesis, we analyzed publicly available chromatin immunoprecipitation sequencing (ChIP-Seq) data for DLX1 in colorectal cancer LoVo cells [25] . By intersecting the genes associated with DLX1 MACS (Model-based Analysis of ChIP-Seq) peaks and the genes downregulated in 22RV1- DLX1 -KO cells, we observed 677 common genes including ALDH1A1 , HNF1A , GATA2 , CDK4 , MYC , WNT5A as the putative transcriptional targets of DLX1 (Supplementary Fig. 3h ). Moreover, DAVID analysis of the common genes revealed downregulation of important biological pathways associated with cancer progression (Supplementary Fig. 3i ). Next, we investigated the expression of PCa associated genes, namely ALDH1A1 [24] , HNF1A [26] , and GATA2 [27] in 22RV1- DLX1 -KO cells, and a significant decrease in their expression compared to control cells was observed (Fig. 2j ). A direct role of DLX1 in upregulating the expression of these genes was established by performing ChIP-qPCR, which confirmed the occupancy of DLX1 on the promoters of ALDH1A1 and HNF1A , while reduced DLX1 enrichment was noted in 22RV1- DLX1 -KO cells (Fig. 2k–m ). Further, decrease in the histone H3 lysine 9 acetylation (H3K9Ac), a transcriptional activation mark at the same sites confirmed DLX1-mediated positive transcriptional regulation (Fig. 2l, m ). Hence, we establish ALDH1A1 and HNF1A as the direct transcriptional targets of DLX1, which are also known to play critical role in stemness, embryonic development, and carcinogenesis [28] , [29] . DLX1 plays pivotal role in tumor growth and metastasis To examine the role of DLX1 in tumorigenesis, we performed mice xenograft experiment by implanting 22RV1- DLX1 -KO or 22RV1-SCR control cells subcutaneously in the flank region of immunodeficient NOD/SCID mice and monitored the animals for tumor growth. A significant decrease in tumor growth with a notable ~80% reduction in tumor burden at the end of the study was observed in the 22RV1- DLX1 -KO cells implanted group compared to the control group (Fig. 3a, b ). To examine spontaneous metastasis, lungs and bone marrow were excised from the xenografted mice and were screened for the presence of human-specific Alu -sequence [30] , [31] . A significant reduction in the number of cells metastasized to the bone marrow and lungs was observed in the 22RV1- DLX1 -KO cells implanted group (Fig. 3c ). We next performed immunohistochemistry (IHC) staining for proliferation (Ki-67) and EMT (Vimentin and E-cadherin) markers on the formalin-fixed paraffin-embedded tumor tissues. A significant reduction in Ki-67 expression, accompanied by reduced Vimentin and increased E-cadherin expression was observed in the DLX1 -KO group compared to control. Moreover, a significant decrease in the expression of DLX1 target, ALDH1A1 was also recorded in DLX1 -KO tumor tissues (Fig. 3d, e ). Notably, immunostaining for ALDH1A1 in the xenograft tumor tissue was heterogenous, indicating random niches of tumor cells having stem cell-like phenotype. Fig. 3: Abrogating DLX1 expression results in tumor regression and reduced metastases. a Mean tumor volume of 22RV1- DLX1 -KO and control SCR cells subcutaneously implanted in NOD/SCID mice ( n = 6, P < 0.0001). b Representative images of the tumors excised at end of the xenograft experiment (top panel). Bar graph showing relative percent reduction in tumor burden. c Bar graphs representing number of cells metastasized to the bone marrow and lungs in xenografted mice as labeled ( n = 5). d Images depicting immunostaining for Ki-67, E-cadherin (E-Cad), Vimentin (VIM), and ALDH1A1 on xenograft tumor sections, images are representative of three tissue samples. Scale bar, 35 µm. e Box plots showing immunostaining quantification of Ki-67, E-Cad, VIM, and ALDH1A1. Quantification was blindly done from 15 random histological fields ( P < 0.0001). f Representative microCT bone images showing horizontal section (top panel) and vertical cross-section (bottom panel) views of the tibia excised from mice ( n = 6) four weeks after intra-medullary tibia injection using 22RV1- DLX1 -KO and control cells. g Same as f , except box plots showing bone architecture parameters analyzed using CTAn software. For panels a , b and c , data represent mean ± SEM. For panels, a Two-way ANOVA, Dunnett’s multiple comparison test b , and c one-way ANOVA, Dunnett’s multiple comparison test; e Unpaired two-tailed Welch’s t -test; g Unpaired two-tailed Student t -test was applied. For panels, e and g Data are presented as box-and-whisker plots indicating median (middle line), 25th and 75th percentile (box) and minimum and maximum values (whiskers). Source data are provided as a Source Data file. Full size image The role of DLX homeobox genes including DLX1 has been established in skeletal development and bone tumors [32] , [33] . Moreover, DLX1 has been reported to play a key role in osteoclastogenesis and bone-resorption [34] , which contributes to osteolytic effects in bone tumors and metastasis [35] . Hence, we next sought to determine the role of DLX1 using an experimental bone metastasis model, wherein intramedullary tibial injection was performed using 22RV1-SCR control and DLX1 -KO cells in athymic NU- Foxn1 nu nude mice. Four weeks post-injection, X-ray scans were taken and subsequently, excised tibia implanted with tumor cells were subjected to micro-computed tomography (microCT), which showed higher bone loss in the control 22RV1-SCR group compared to DLX1 -KO (Fig. 3f and Supplementary Fig 3j ). Further, we examined the bone morphometric parameters of the metaphysis region of the tibia from both groups using CTAn (CT-Analyser) software. 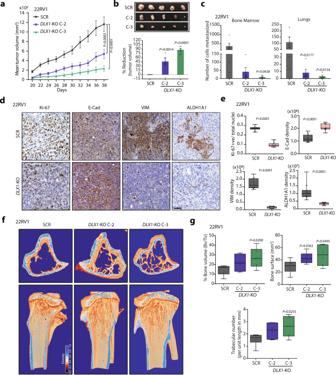Fig. 3: Abrogating DLX1 expression results in tumor regression and reduced metastases. aMean tumor volume of 22RV1-DLX1-KO and control SCR cells subcutaneously implanted in NOD/SCID mice (n= 6,P<0.0001).bRepresentative images of the tumors excised at end of the xenograft experiment (top panel). Bar graph showing relative percent reduction in tumor burden.cBar graphs representing number of cells metastasized to the bone marrow and lungs in xenografted mice as labeled (n= 5).dImages depicting immunostaining for Ki-67, E-cadherin (E-Cad), Vimentin (VIM), and ALDH1A1 on xenograft tumor sections, images are representative of three tissue samples. Scale bar, 35 µm.eBox plots showing immunostaining quantification of Ki-67, E-Cad, VIM, and ALDH1A1. Quantification was blindly done from 15 random histological fields (P< 0.0001).fRepresentative microCT bone images showing horizontal section (top panel) and vertical cross-section (bottom panel) views of the tibia excised from mice (n= 6) four weeks after intra-medullary tibia injection using 22RV1-DLX1-KO and control cells.gSame asf, except box plots showing bone architecture parameters analyzed using CTAn software. For panelsa,bandc, data represent mean ± SEM. For panels,aTwo-way ANOVA, Dunnett’s multiple comparison testb, andcone-way ANOVA, Dunnett’s multiple comparison test;eUnpaired two-tailed Welch’st-test;gUnpaired two-tailed Studentt-test was applied. For panels,eandgData are presented as box-and-whisker plots indicating median (middle line), 25th and 75th percentile (box) and minimum and maximum values (whiskers). Source data are provided as a Source Data file. Interestingly, tibia implanted with DLX1 -KO cells showed an increase in bone volume fraction (Bv/Tv), bone surface (BS), and trabecular number (TN) compared to tibia in the control group, thus signifying the presence of bone loss and destruction of bone architecture in 22RV1-SCR control group (Fig. 3g ). Taken together, these findings provide a comprehensive understanding of DLX1-mediated oncogenicity and its possible role in PCa associated bone metastases. Elevated ERG and AR levels show positive association with DLX1 expression Overexpression of ETS transcription factor, ERG owing to TMPRSS2–ERG gene rearrangement is considered an early event in ∼ 50% of PCa cases [1] , thus we next examined the association of DLX1 with ERG using the publicly available TCGA-PRAD [36] cohort. Stratification of the clinical genomic data of PCa patients ( n = 498) based on the expression of ERG revealed that most of the cases with higher ERG levels also exhibit increased expression of DLX1 transcript (Fig. 4a ). Next, using the UALCAN cancer OMICS database [37] we analyzed the overall survival probability of patients with varying expression of DLX1 and its association with the well-known seven molecular PCa subtypes defined by TCGA [36] . Notably, TMPRSS2-ERG fusion-positive patients with higher levels of DLX1 experienced lower survival probability compared to fusion-positive patients with low/medium DLX1 expression (Supplementary Fig. 4a ), indicating the possible existence of oncogenic cooperativity between DLX1 and ERG. Furthermore, a significant positive correlation between DLX1 and ERG expression was observed in both MSKCC [38] and TCGA-PRAD cohorts (Supplementary Fig. 4b, c ). Fig. 4: Elevated ERG and AR correlates with higher DLX1 levels representing advanced-stage aggressive disease. a Heatmap showing TCGA-PRAD RNA-Seq data for ERG and DLX1 expression in primary PCa specimens ( n = 498). Shades of red and blue represent the log 2 (norm_count+1) value. b Representative core of PCa tissue microarray (TMA) showing RNA in situ hybridization (RNA-ISH) scoring pattern for DLX1 in 144 PCa patient specimens, score 0 represents DLX1 negative, score 1 signifies low DLX1, score 2, and score 3 represents medium and high DLX1 expression, respectively. Scale bar, 50 µm. c Bar plot showing percentage of patients negative (DLX1–) and positive (DLX1+) for DLX1 expression based on the scoring pattern ( P < 0.0001). d Same as b except Immunohistochemistry (IHC) for ERG (top panel) and RNA-ISH for DLX1 (bottom) in 144 PCa patient tissue specimens. e Bar plot showing percentage of patients with varying DLX1 expression in ERG-positive (ERG+) and -negative (ERG–) PCa cases ( P < 0.0001). f Same as e except an association between ERG and DLX1 expression status and Gleason scores of PCa patients ( P = 0.0003). g Same as b except representative tumor cores showing IHC for AR, ERG, and RNA-ISH for DLX1 representing AR+/ERG+/DLX1+ status in 144 PCa patient tissue specimens. h Same as g except for representative AR + /ERG−/DLX1+ patient in TMA containing 144 PCa specimens. i Bar plot depicting percentage of patients with positive and negative DLX1 expression in AR + /− and ERG + /− respective background. Patients showing low, medium, and high DLX1 expression categorized as DLX1-positive ( P < 0.0001). j Contingency table for the AR and DLX1 status in TMA patient specimens. 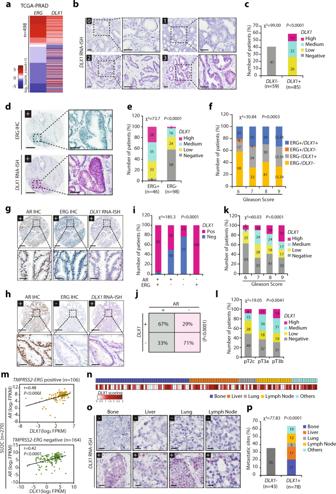Fig. 4: Elevated ERG and AR correlates with higher DLX1 levels representing advanced-stage aggressive disease. aHeatmap showing TCGA-PRAD RNA-Seq data forERGandDLX1expression in primary PCa specimens (n= 498). Shades of red and blue represent the log2(norm_count+1) value.bRepresentative core of PCa tissue microarray (TMA) showing RNA in situ hybridization (RNA-ISH) scoring pattern forDLX1in 144 PCa patient specimens, score 0 represents DLX1 negative, score 1 signifies low DLX1, score 2, and score 3 represents medium and high DLX1 expression, respectively. Scale bar, 50 µm.cBar plot showing percentage of patients negative (DLX1–) and positive (DLX1+) forDLX1expression based on the scoring pattern (P< 0.0001).dSame asbexcept Immunohistochemistry (IHC) for ERG (top panel) and RNA-ISH forDLX1(bottom) in 144 PCa patient tissue specimens.eBar plot showing percentage of patients with varyingDLX1expression in ERG-positive (ERG+) and -negative (ERG–) PCa cases (P< 0.0001).fSame aseexcept an association between ERG andDLX1expression status and Gleason scores of PCa patients (P= 0.0003).gSame asbexcept representative tumor cores showing IHC for AR, ERG, and RNA-ISH forDLX1representing AR+/ERG+/DLX1+ status in 144 PCa patient tissue specimens.hSame asgexcept for representative AR + /ERG−/DLX1+ patient in TMA containing 144 PCa specimens.iBar plot depicting percentage of patients with positive and negativeDLX1expression in AR + /− and ERG + /− respective background. Patients showing low, medium, and highDLX1expression categorized as DLX1-positive (P< 0.0001).jContingency table for the AR andDLX1status in TMA patient specimens.P-value denotes Fisher’s exact test (P< 0.0001).kBar plot showing association betweenDLX1expression and Gleason scores of tumor specimens (P< 0.0001).lSame ask, except association ofDLX1expression with tumor stage (P= 0.0041).mCorrelation plot of AR andDLX1using Stand Up To Cancer (SU2C) dataset by categorizing patients asTMPRSS2-ERGpositive (top panel) and negative samples (bottom panel).P-value was calculated using two-tailed test with 95% confidence interval (P< 0.0001).nHeatmap showingDLX1levels in tumor specimens representing distant metastatic sites of metastatic CRPC patients.oSame asnexcept for RNA-ISH forDLX1expression in TMA containing 121 mCRPC biospecimens collected from various metastatic sites. Scale bar, 25 µm.pBar plot showing DLX1 expression in percent metastatic sites from CRPC patients same asn(P< 0.0001). For panelsd,g, andhscale bars are represented as 300 µm for the entire core and 50 µm for the inset image. For panels,c, e,f,i,k,l, andpP-value were calculated using Chi-Square test. Source data are provided as a Source Data file. P -value denotes Fisher’s exact test ( P < 0.0001). k Bar plot showing association between DLX1 expression and Gleason scores of tumor specimens ( P < 0.0001). l Same as k , except association of DLX1 expression with tumor stage ( P = 0.0041). m Correlation plot of AR and DLX1 using Stand Up To Cancer (SU2C) dataset by categorizing patients as TMPRSS2-ERG positive (top panel) and negative samples (bottom panel). P -value was calculated using two-tailed test with 95% confidence interval ( P < 0.0001). n Heatmap showing DLX1 levels in tumor specimens representing distant metastatic sites of metastatic CRPC patients. o Same as n except for RNA-ISH for DLX1 expression in TMA containing 121 mCRPC biospecimens collected from various metastatic sites. Scale bar, 25 µm. p Bar plot showing DLX1 expression in percent metastatic sites from CRPC patients same as n ( P < 0.0001). For panels d , g , and h scale bars are represented as 300 µm for the entire core and 50 µm for the inset image. For panels, c, e , f , i , k , l , and p P -value were calculated using Chi-Square test. Source data are provided as a Source Data file. Full size image To further confirm these findings, we performed IHC, and RNA in situ hybridization (RNA-ISH) for ERG and DLX1 expression, respectively using a tissue microarray (TMA) comprising 144 PCa patient specimens, and all but three of these patients were hormone naïve. The RNA-ISH staining patterns for DLX1 were classified into four levels ranging from the score of 0–3, nearly ~60% of the patients were found positive for DLX1 expression ranging from low to high (Fig. 4b, c ). Specimens stained for ERG were stratified into ERG positive (ERG+) and negative (ERG-) categories (Supplementary Fig. 4d ). In agreement with our in silico analysis, 44 out of 46 TMPRSS2-ERG fusion-positive cases (~96%) showed positive staining for DLX1 expression (Fig. 4d, e and Supplementary Fig. 4e ), wherein ~28% patients showed a high score for DLX1 ( DLX1 Hi , score 3), ~35% patients with moderate ( DLX1 Me , score 2) and ~33% patients with lower DLX1 expression ( DLX1 Lo , score 1) (Fig. 4e ), suggesting a possible role of ERG in DLX1 regulation. While ~42% ERG-negative tumors also show DLX1 expression, indicating the involvement of ERG-independent pathway in its regulation (Supplementary Fig. 4e ). In terms of clinical staging, the percentage of tumors stained positive for both ERG and DLX1 substantially increase from ~21% in low Gleason score (GS6) to ~33% in high Gleason score disease (GS9), similarly tumors stained positive only for DLX1 expression (ERG–/DLX1+) also exhibit higher Gleason score (Fig. 4f ). Thus, suggesting that the majority of the PCa patients harboring higher DLX1 with/without ERG expression (ERG+/DLX1+ and ERG-/DLX1+) are associated with advanced-stage disease. Next, we explored the status of AR expression in these patient samples and examined its correlation with DLX1 expression. To achieve this, we performed IHC staining for AR on the same TMA and stratified the specimens as AR-positive (AR+) and negative (AR–) based on the staining intensity (Supplementary Fig. 4f ). Next, the specimens categorized as AR+ were further examined for the presence or absence of ERG expression and/or DLX1 expression by RNA-ISH (Fig. 4g, h ). Interestingly, we found that ~95% of the patients (42 out of 44) positive for AR and ERG (AR+/ERG+) showed DLX1 expression, similarly ~50% of the AR+/ERG– patients (36 out of 72) were also positive for DLX1 (Fig. 4i ), while this percentage decreased (~23%) for the patients (6 out of 26) whose tumors were negative for both AR and ERG. However, only two patients which were AR-negative and ERG-positive showed DLX1 expression (Fig. 4i ). This data was re-examined by stratifying patients’ specimens based on AR expression, and we found that ~67% of the AR+ patients also exhibit DLX1 expression (Fig. 4j ). While ~29% of the AR– patients show DLX1 expression, indicating a possible role of some other regulatory factor(s) contributing to DLX1 upregulation (Fig. 4j ). Moreover, DLX1 level alone gradually increased as a function of disease stage; ~37% positive in GS6 disease to ~67% positive in GS9 disease (Fig. 4k ), similarly, ~51% in pT2c (pathologic tumor 2c) to 69% in pT3b stage (Fig. 4l ). Providing the association of DLX1 with advanced-stage disease, we analyzed Stand Up to Cancer (SU2C) metastatic PCa dataset publicly available on cBioPortal for the expression of DLX1 and its correlation with AR and ERG [39] . A significant positive correlation between AR and DLX1 expression was observed in metastatic PCa patients irrespective of TMPRSS2-ERG fusion status (Fig. 4m ). Further, we performed RNA-ISH for DLX1 in a metastatic PCa TMA comprising 121 metastatic sites collected from 45 patients (Fig. 4n, o ). We found that ~64% of total metastatic sites showed DLX1 expression, of these 21% belonged to bone, 17% to liver, 5% to lung, 12% to lymph node, and 10% to other organ sites (Fig. 4p ). Together, our data suggest a role of DLX1 in aggressive and metastatic PCa and indicate a plausible oncogenic cooperativity between DLX1, ERG, and AR in the progression of this disease. ERG regulates DLX1 in TMPRSS2-ERG fusion-positive prostate cancer Since we found a strong association between ERG and DLX1 expression in several independent PCa cohorts, we next sought to investigate the role of ERG in transcriptional regulation of DLX1 . Thus, we analyzed publicly available ERG ChIP-Seq dataset in VCaP ( TMPRSS2-ERG fusion-positive) cells [40] , [41] , and an increased enrichment of ERG on the DLX1 promoter was observed, while it was reduced in ERG depleted cells (Fig. 5a ). Furthermore, enrichment of ERG on the DLX1 promoter was also observed in ectopic ERG overexpressing RWPE1 cells [42] (Fig. 5a ). Next, we scanned ~1 kb upstream and 500 bp downstream region to the transcription start site (TSS) of DLX1 for the presence of probable ERG binding motif (EBM), and putative ERG binding sites namely, EBM1 (P1) and EBM2 (P2) were noticed (Fig. 5b ). Next, our ChIP-qPCR data confirmed the significant recruitment of ERG at these EBMs on the DLX1 promoter in VCaP cells (Fig. 5b ). To confirm whether ERG occupancy is associated with transcriptionally active chromatin, we examined the presence of transcriptional activation marks, and a marked enrichment of H3K9Ac along with RNA polymerase II (RNA-Pol II) was observed (Fig. 5b ). PLAU , an ERG target gene was used as a positive control. In agreement with this, ectopic ERG overexpression in RWPE1 cells (RWPE1-ERG) resulted in upregulation of DLX1 both at the transcript and protein levels (Fig. 5c ). Furthermore, isogenic RWPE1 cells were examined for the ERG-mediated activation of the DLX1 promoter by luciferase-based DLX1 promoter reporter assay. As speculated, a significant increase in the reporter activity was observed in RWPE1-ERG cells transfected with a wild-type DLX1 promoter reporter, while no significant change in the luciferase activity with mutated EBMs was observed (Fig. 5d ). Fig. 5: DLX1 is a transcriptional target of ERG in TMPRSS2-ERG positive prostate cancer. a Chromatin immunoprecipitation-sequencing (ChIP-Seq) data depicting ERG enrichment at the DLX1 promoter in the indicated cell lines from GEO databases (GSE98809, GSE110655, and GSE37752). b Schema showing chromosomal location of the ERG binding motifs (EBM) onto DLX1 promoter selected for ChIP-qPCR (top panel). ChIP-qPCR data showing recruitment of ERG, histone H3 lysine 9 acetylation (H3K9Ac), and RNA-polymerase II (RNA-Pol II) at the DLX1 and PLAU promoters. c Q-PCR (left panel) and immunoblot (right panel) data showing the expression of ERG and DLX1 in RWPE1 cells overexpressing ERG ( P < 0.0001). d Schema showing site-directed mutagenesis of DLX1 promoter cloned upstream of luciferase gene, nucleotides in red were mutated (top). Luciferase reporter assay indicating wild-type (WT) and mutant (Mut) DLX1 promoter-driven reporter activity (bottom panel) in ERG overexpressing and control RWPE1 cells ( P < 0.0001). e Q-PCR data showing relative expression of target genes in VCaP cells stimulated with 10 nM R1881 at the indicated time points. f Same as e , except immunoblot data. g Schematic diagram depicting ERG-mediated transcriptional regulation of DLX1 and plausible role of AR in DLX1 regulation. h ChIP-Seq data (GSE28951) showing recruitment of AR and ERG on the DLX1 enhancer and promoter regions respectively, in R1881-stimulated VCaP cells. i ChIP-Seq data (GSE70079) showing enrichment of AR at the DLX1 putative enhancer in the normal prostate ( n = 6) and PCa ( n = 13) tissue specimens. KLK3 represents positive control. Data shown from three biologically independent samples ( n = 3). Data represent mean ± SEM. For panels, b Unpaired two-tailed Welch’s t -test; c and d Two-way ANOVA Sidak’s multiple comparison test; e Two-way ANOVA, Dunnett’s multiple comparison test was applied. Source data are provided as a Source Data file. Full size image Since AR signaling is known to drive the expression of ERG in TMPRSS2-ERG fusion - positive background, we next examined the effect of synthetic androgen methyltrienolone (R1881) on the expression of DLX1 in VCaP cells. Notably, ~2-fold increase in DLX1 expression both at the transcript and protein levels was observed in R1881-stimulated VCaP cells (Fig. 5e, f ). PSA was included as a positive control for androgen stimulation. Next, we tested whether AR also plays a direct role in the transcriptional regulation of DLX1 (Fig. 5g ). Thus, to ascertain this, we analyzed ChIP-Seq datasets (GSE28951) [2] for AR and ERG in R1881-stimulated VCaP cells. Notably, a strong binding of AR on the third exon (chr2:172,661,000-172,662,500) of DLX1 was observed in R1881-stimulated VCaP cells (Fig. 5h ). On similar lines, several studies revealed the presence of exonic enhancers (eExons) which can act as a regulatory element for the nearby genes or the host gene on which they reside [43] , [44] . Hence, we propose that the presence of AREs at the third exon may act as a putative enhancer region in the transcriptional regulation of DLX1 . We further examined the binding of AR on the DLX1 gene using publicly available dataset (GSE70079) [45] comprising normal and PCa specimens, and a remarkable enrichment of AR was observed on the putative enhancer element of the DLX1 in PCa specimens (Fig. 5i ). Conclusively, we show that ERG directly gets recruited on the DLX1 promoter thereby regulating its expression in TMPRSS2-ERG positive cases. Our findings also imply the potential role of AR signaling in mediating DLX1 expression in PCa. AR regulates DLX1 expression in prostate cancer Considering an association between AR and DLX1 expression in PCa specimens and AR occupancy at the DLX1 enhancer region, we next sought to examine the role of androgen signaling in the regulation of DLX1 . Previously, presence of distinct AR binding sites (ARBS) were reported in tumor tissues than in normal prostatic tissue [45] . Furthermore, DLX1 was found in the top ten upregulated genes in TCGA-PRAD dataset, which harbor tumor-specific ARBS in the neighboring 50 kb region (Supplementary Fig. 5a ). To further validate the AR binding on the putative enhancer of DLX1 , we performed ChIP-qPCR using R1881-stimulated VCaP cells, identifying a significant enrichment of AR on the DLX1 enhancer, which was disrupted upon anti-androgen enzalutamide (Enza) treatment (Fig. 6a ). The ARBS of KLK3 was used as a positive control (Supplementary Fig. 5b ). Further, we also examined the effect of another anti-androgen, EPI-001 on DLX1 expression, a selective AR inhibitor that impedes transactivation of the amino-terminal domain (NTD) of AR thereby abrogating AR-V7 mediated transcriptional activity [46] . As speculated, treatment of VCaP cells with Enza and EPI-001 abrogated R1881-induced DLX1 expression, implicating the role of AR in transcriptional regulation of DLX1 (Fig. 6b ). Since FOXA1 is a known pioneer TF and a coactivator of AR [47] , we next investigated the occupancy of FOXA1 at the DLX1 putative enhancer region. Importantly, ChIP-qPCR in VCaP cells show FOXA1 enrichment on the same locus, signifying the recruitment of AR transcriptional complex on the putative enhancer region of DLX1 (Fig. 6c ). Similarly, ChIP-Seq analysis (GSE56086) [48] also revealed FOXA1 binding at the same locus (chr2:172,661,000-172,662,500) as occupied by AR (Supplementary Fig. 5c ). Since AR and ERG interaction as a coregulatory TF is known to regulate the expression of common target genes [3] , [49] , we examined the probable co-interaction of ERG and AR at the DLX1 promoter by performing re-ChIP experiment (Fig. 6d ). As anticipated, ChIP using ERG antibody followed by pulldown using an AR antibody showed significant enrichment of AR and ERG at the DLX1 promoter, thus confirming their interaction through the promoter-enhancer region (Fig. 6d ). CUTL2 , an AR-ERG co-regulated gene was used as a positive control. To further validate the plausible chromatin interaction at the DLX1 genomic region, we analyzed the 3D-chromatin landscape of RNA-Pol II in VCaP cells using ChIA-PET dataset (GSE121020) [50] . The integrative analysis of RNA-Pol II-associated peaks along with ChIP-Seq data of DLX1 regulating TFs in PCa was performed. Consistent with our findings, the RNA-Pol II ChIA-PET data confirmed the promoter-enhancer interaction at the DLX1 gene, which also indicated the binding of ERG, AR, and FOXA1 transcription factors (Fig. 6e ). Owing to the promoter-enhancer interaction at DLX1 gene loci and ERG occupancy at DLX1 enhancer region in ChIP-Seq data (Fig. 6e ), we carried out ChIP-qPCR for ERG at the DLX1 enhancer region. As expected, we observed notable enrichment of ERG at the enhancer region of DLX1 (Fig. 6f ). Remarkably, siRNA-mediated knockdown of these regulatory factors namely, ERG , AR and FOXA1 in VCaP cells (Supplementary Fig. 5d ) resulted in reduced DLX1 expression across all siRNA conditions (Fig. 6g, h ). Also, pronounced decrease in the level of DLX1 was achieved by concurrent silencing of all the three key regulators ( ERG , AR , and FOXA1 ), thereby indicating the transcriptional interplay between these factors. Since the downregulation of FOXA1 is known to reprogram AR binding cistrome in PCa [45] , we next examined if silencing FOXA1 in VCaP cells redistributes binding of AR at DLX1 enhancer region. Hence, we performed ChIP-qPCR for the AR occupancy in FOXA1- silenced VCaP cells and reduced AR enrichment at the DLX1 enhancer region was observed, which was concordant with decrease in FOXA1 occupancy at these sites (Fig. 6i and Supplementary Fig. 5e ). Collectively, our results suggest ERG and AR-mediated transcriptional co-regulation of DLX1 in TMPRSS2-ERG fusion-positive cells. Furthermore, shRNA-mediated AR knockdown in castration-resistant and TMPRSS2-ERG fusion-negative, C4-2 cells also showed decrease in DLX1 expression (Supplementary Fig. 5f ). 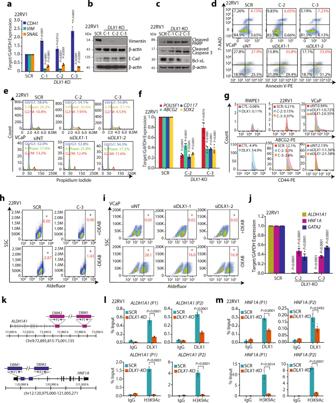Moreover, upon androgen stimulation, enrichment of AR and FOXA1 was observed in TMPRSS2-ERG fusion-negative 22RV1 cells, suggesting the significance of AR signaling in transcriptional regulation of DLX1 in an ERG-independent manner (Fig. 6j ). Fig. 2: Genetic ablation ofDLX1inhibits oncogenic properties. aQ-PCR data showing expression of EMT markers in 22RV1-DLX1-KO and control SCR cells.bImmunoblots showing vimentin and E-cadherin using same cells asa. β-actin was used as loading control.cSame asbexcept for cleaved PARP, cleaved Caspase-3 and Bcl-xL.dFlow cytometry-based apoptosis assay using 22RV1-DLX1-KO and control cells (top panel) andDLX1-silenced VCaP cells (bottom panel).eFlow cytometry data for cell cycle distribution using same cells as ind.fQ-PCR data for stem cell markers using same cells asd.gFlow cytometry data depicting ABCG2 (top panel) and CD44 (bottom panel) expression in DLX1 overexpressing RWPE1 cells, 22RV1-DLX1-KO, andDLX1-silenced VCaP cells.hFluorescence intensity of catalyzed ALDH substrate in 22RV1-DLX1-KO and control cells. Marked windows show ALDH1 + percent cell population.iSame ash, except forDLX1silenced VCaP cells.jQ-PCR data showing expression of target genes in 22RV1-DLX1-KO and control cells(P< 0.0001).kSchema showing the chromosomal location ofDLX1binding motif (DBM1/2) at theALDLH1A1(top) andHNF1A(bottom) promoters.lChIP-qPCR data of DLX1 (top panel) and H3K9Ac (bottom panel) onALDH1A1in 22RV1-DLX1-KO and SCR control cells (P< 0.0001).mSame as inlexcept for theHNF1Apromoter. Data shown from three biologically independent samples (n= 3). Data represent mean ± SEM. For panels,a,f, andjTwo-way ANOVA, Dunnett’s multiple comparison test;l,mTwo-way ANOVA Turkey’s multiple comparison test was applied. Source data are provided as a Source Data file. Fig. 6: AR and AR-V7 regulate DLX1 expression in both ERG-dependent and -independent manners. a Schematic showing the androgen response elements (AREs) at the DLX1 putative enhancer (top panel). ChIP-qPCR data (bottom panel) depicting AR recruitment at the DLX1 putative enhancer in R1881 (10 nM) stimulated VCaP cells in the presence or absence of Enzalutamide (Enza, 10 µM) ( P < 0.0001). b Immunoblot (top panel) and Q-PCR (bottom panel) data showing relative expression of target genes in VCaP cells under similar culture conditions as indicated. c ChIP-qPCR data depicting FOXA1 recruitment at the DLX1 putative enhancer in R1881 (10 nM) stimulated VCaP. d Schematic representation showing the possible interaction between ERG and AR on the DLX1 promoter (top panel). Re-ChIP data showing co-enrichment of AR and ERG on EBM at the DLX1 promoter (bottom panel). e Integrated genome view of 3D-chromatin structure and binding of transcription factors at the genomic and nearby region of DLX1 . f Bar plots depicting ChIP-qPCR data for ERG occupancy at the DLX1 enhancer region. g Q-PCR data showing relative expression of DLX1 in siRNA-mediated ERG , AR, and/or FOXA1 -silenced VCaP cells. h Same as g except immunoblot data. i ChIP-qPCR data showing enrichment of AR (top panel) and FOXA1 (bottom panel) in siRNA-mediated FOXA1 -silenced VCaP cells . j ChIP-qPCR data depicting AR (top panel) and FOXA1 (bottom panel) enrichment at the DLX1 putative enhancer in 22RV1 cells stimulated with R1881 (10 nM) for 16 h. KLK3 shown as a positive control. k Relative expression of KLK3 and DLX1 in doxycycline (Dox) induced AR-V7 overexpressing LNCaP cells treated with R1881 (10 nM). For induction, 40 ng/ml of Dox or vehicle control was used for 24 and 48 h. l Immunoblots showing the expression of AR-FL, AR-V7, DLX1, and PSA using same cells as k . β-actin used as loading control. m Q-PCR data showing DLX1 and KLK3 expression in LNCaP AR-V7 cells under similar culture conditions as mentioned at 48-h time point. Data shown from three biologically independent samples ( n = 3). Data represent mean ± SEM. For panels, a , b Two-way ANOVA Sidak’s multiple comparison test; f Unpaired two-tailed Welch’s t -test; g One-way ANOVA, Dunnett’s multiple comparison test; c , i , j , m Two-way ANOVA, Tukey’s multiple comparisons; k Two-way ANOVA, Dunnett’s multiple comparison test was applied. Source data are provided as a Source Data file. Full size image Having established the higher DLX1 expression in CRPC cases and deciphering a substantial role of full-length AR in modulating its expression, we considered the possible involvement of AR-V7, an AR splice variant in transcriptional regulation of DLX1. Intriguingly, ChIP-Seq analysis for AR-V7 specific binding in 22RV1 cells revealed remarkable enrichment of AR-V7 at the putative enhancer region of DLX1 (Supplementary Fig. 5g ). Moreover, analysis of publicly available RNA-Seq data (GSE94013) [51] shows a significant reduction in DLX1 transcript upon silencing AR-V7 or AR-FL in 22RV1 cells (Supplementary Fig. 5h ) suggesting the role of AR-V7 in DLX1 regulation. Furthermore, using an inducible expression system for AR-V7, we generated LNCaP cells that can express both AR-FL and AR-V7, which mimics the clinical state of the majority of PCa patients with resistance to enzalutamide or abiraterone [52] . In these genetically engineered LNCaP cells, the expression levels of AR-FL and AR-V7 can be induced by treating them with R1881 and doxycycline (dox), respectively (Fig. 6k ). In line with this, both AR-FL, as well as AR-V7 expression, led to increased expression of DLX1 transcript and protein levels (Fig. 6k, l ). As we conjecture, treating LNCaP AR-V7 cells with AR antagonists (enzalutamide or EPI-001) in the presence of R1881 or dox abrogated AR-FL and AR-V7 mediated increase in DLX1 expression (Fig. 6m ). Taken together, our findings suggest a role of AR-FL and AR-V7 in the transcriptional regulation of DLX1 in ERG-dependent as well as -independent manner. These findings also highlight the critical role of AR-V7 in the transcriptional regulation of DLX1 , thereby resonating with relatively high DLX1 expression in PCa patients with advanced-stage disease and higher Gleason score. BETi attenuates DLX1 expression and its oncogenic properties Having established ERG and AR signaling mediated transcriptional regulation of DLX1 , we next explored the therapeutic strategies to target this regulatory circuitry. Since the utility of BETi, namely JQ1 and I-BET762 has been shown to inhibit aberrant AR signaling and the localization of BRD4 to AR target genes [12] , we sought to investigate the ability of JQ1 in impeding the transcriptional regulators of DLX1 , namely ERG and AR. Using ChIP-Seq dataset (GSE55064) [12] , we examined the recruitment of ERG on DLX1 promoter following BETi treatment in VCaP cells. Interestingly, a remarkable decrease in the enrichment of ERG was observed in JQ1 treated VCaP cells compared to control (Fig. 7a ). Moreover, the presence of H3K27Ac marks indicates active DLX1 promoter in the control VCaP cells, and PLAU , a known ERG target gene was used as a positive control (Fig. 7a ). Further, these results were confirmed by ChIP-qPCR for ERG using JQ1 treated VCaP cells, and a similar trend was observed (Fig. 7b ). We also looked for change in the DLX1 expression in JQ1 treated VCaP cells, and a significant decrease in its expression was observed (Supplementary Fig. 6a, b ). To examine whether JQ1 can inhibit ERG-mediated DLX1 expression, stable RWPE1-ERG cells were treated with JQ1, and a reduced DLX1 expression was observed, thereby confirming the efficacy of JQ1 in inhibiting ERG-mediated transcriptional regulation of DLX1 (Supplementary Fig. 6c ). Considering ERG-independent role of AR in DLX1 regulation, we next treated C4-2, C4-2B, and 22RV1 cells with JQ1, and as speculated a significant reduction in the DLX1 expression was noted (Supplementary Fig. 6d ). Furthermore, VCaP and C4-2 cells treated with JQ1 showed a significant decrease in cell proliferation compared to vehicle control (Supplementary Fig. 6e ). In addition, we performed GSEA analysis of publicly available RNA-Seq data of JQ1 treated 22RV1 cells (GSE162564) using DLX1 putative target (Supplementary Fig. 3h ) and observed enrichment of DLX1 target genes in control cells (Supplementary Fig. 6f ). These data suggest downregulation of DLX1 putative target genes resulting in decreased oncogenic effect upon JQ1 treatment. Fig. 7: BET inhibitor alone or in combination with Enzalutamide downregulates DLX1 expression and mitigates its oncogenic properties. a ChIP-Seq data (GSE55064) showing ERG enrichment on DLX1 promoter in VCaP cells treated with JQ1 or vehicle control for 24 h. H3K27Ac represents active promoter in untreated cells. PLAU used as a positive control. b ChIP-qPCR data showing relative ERG enrichment on DLX1 promoter in VCaP cells treated with JQ1 (0.5 µM) for 48 h ( P < 0.0001). c Q-PCR data showing relative expression of target genes in VCaP cells treated with Enza (10 µM), JQ1 (0.5 µM) alone or in combination for 48 h. KLK3 used as a positive control for JQ1 treatment. d Same as c except immunoblot. β-actin was used as loading control. e Same as c except 22RV1 cells. f Same as e except immunoblot ( P < 0.0001). g Cell proliferation assay in VCaP cells treated with drug conditions as mentioned in c . h Same as g except 22RV1 cells ( P < 0.0001). i Same as g except 42D ENZ R cells ( P < 0.0001). j Boyden Chamber Matrigel migration assay in VCaP cells using same treatment conditions as c . Inset shows representative image of the migrated cells (scale bar 30 µm). k Same as j except 22RV1 cells (scale bar 30 µm, P < 0.0001). l Same as j except Enza-resistant, 42D ENZ R cells (scale bar 30 µm, P < 0.0001). m Fluorescence intensity of the catalyzed ALDH substrate in VCaP cells under same treatment conditions as c . Marked windows show ALDH1+ percent cell population. 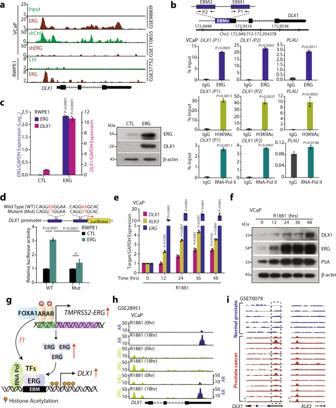Fig. 5:DLX1is a transcriptional target of ERG inTMPRSS2-ERGpositive prostate cancer. aChromatin immunoprecipitation-sequencing (ChIP-Seq) data depicting ERG enrichment at theDLX1promoter in the indicated cell lines from GEO databases (GSE98809, GSE110655, and GSE37752).bSchema showing chromosomal location of the ERG binding motifs (EBM) ontoDLX1promoter selected for ChIP-qPCR (top panel). ChIP-qPCR data showing recruitment of ERG, histone H3 lysine 9 acetylation (H3K9Ac), and RNA-polymerase II (RNA-Pol II) at theDLX1andPLAUpromoters.cQ-PCR (left panel) and immunoblot (right panel) data showing the expression of ERG and DLX1 in RWPE1 cells overexpressing ERG (P< 0.0001).dSchema showing site-directed mutagenesis ofDLX1promoter cloned upstream of luciferase gene, nucleotides in red were mutated (top). Luciferase reporter assay indicating wild-type (WT) and mutant (Mut)DLX1promoter-driven reporter activity (bottom panel) in ERG overexpressing and control RWPE1 cells (P< 0.0001).eQ-PCR data showing relative expression of target genes in VCaP cells stimulated with 10 nM R1881 at the indicated time points.fSame ase, except immunoblot data.gSchematic diagram depicting ERG-mediated transcriptional regulation ofDLX1and plausible role of AR in DLX1 regulation.hChIP-Seq data (GSE28951) showing recruitment of AR and ERG on theDLX1enhancer and promoter regions respectively, in R1881-stimulated VCaP cells.iChIP-Seq data (GSE70079) showing enrichment of AR at theDLX1putative enhancer in the normal prostate (n= 6) and PCa (n= 13) tissue specimens.KLK3represents positive control. Data shown from three biologically independent samples (n= 3). Data represent mean ± SEM. For panels,bUnpaired two-tailed Welch’st-test;canddTwo-way ANOVA Sidak’s multiple comparison test;eTwo-way ANOVA, Dunnett’s multiple comparison test was applied. Source data are provided as a Source Data file. n Same as m except 22RV1 cells. o Same as m except 42D ENZ R cells. p Bar plot showing number of spheres formed in prostatosphere assay using VCaP under same treatment conditions as c . Inset shows representative image of the spheres formed (scale bar 100 µm). q Q-PCR data for the DLX1 expression using RNA isolated from VCaP prostatospheres. Data shown from three biologically independent samples ( n = 3). Data represent mean ± SEM. For panels b , c , e two-way ANOVA, Tukey’s multiple comparison test; g , h , i One-way ANOVA, Dunnett’s multiple comparison test; j – l , p , q One-way ANOVA, Tukey’s multiple comparison was applied. Source data are provided as a Source Data file. Full size image Recent preclinical and phase Ib/IIa clinical studies reported the efficacy of BET inhibitors in combination with anti-androgens in CRPC patients [13] , [53] . Hence, we examined whether JQ1 along with Enza could be effective in attenuating DLX1 expression and its oncogenic properties. Thus, we treated VCaP cells ( TMPRSS2-ERG positive) with JQ1 alone or with Enza and examined the expression of DLX1 and its target genes. Intriguingly, we observed ~60% reduction in DLX1 expression as well as a concomitant decrease in the expression of DLX1 target genes, namely ALDH1A1 and HNF1A in JQ1 treated VCaP cells compared to vehicle control (Fig. 7c ). Although this effect was more pronounced (~90%) when VCaP cells were treated with JQ1 and Enza combination (Fig. 7c, d ). Further, to investigate the JQ1 inhibitory effect in ERG-independent background, we treated castrate-resistant 22RV1 cells (ERG-negative) with both BETi and Enza. As speculated, a similar inhibitory effect in the expression of DLX1 , ALDH1A1 , and HNF1A was observed with JQ1 and/or Enza, indicating the absence of combinatorial additive effects as in case of VCaP cells (Fig. 7e, f ). Nonetheless, PCa cells treated with Enza alone resulted in increased HNF1A expression which corroborates with the previous reports [26] . To investigate the efficacy of JQ1 in anti-androgen resistant cell line model, we performed similar experiments with enzalutamide-resistant 42D ENZ R cells (DLX1-positive and ERG-negative). As speculated, 42D ENZ R cells showed decrease in DLX1 expression in response to JQ1 treatment alone (Supplementary Fig. 6g, h ). Further, we examined the effect of these drugs on the oncogenic properties in both ERG-dependent and -independent backgrounds, observing a marked reduction in cell proliferation rates of VCaP, 22RV1, and 42D ENZ R cells treated with JQ1 alone as anticipated. Combinatorial treatment with JQ1 and Enza exhibited a remarkable reduction in VCaP cell proliferation, but no such effect was noticed in 22RV1 and 42D ENZ R cells (Fig. 7g–i ). Likewise, treatment of VCaP, 22RV1, and 42D ENZ R cells with JQ1 and/or Enza showed a decrease in the cell migratory and foci forming abilities, although this inhibitory effect was more evident in VCaP cells treated with the drug combination (Fig. 7j–l and Supplementary Fig. 6i–k ). Since we showed ALDH1A1 as one of the DLX1 target genes, we next analyzed ALDH activity in response to JQ1 alone or combined with Enza in VCaP, 22RV1, and 42D ENZ R cells using flow cytometry-based assay. Interestingly, reduced levels of ALDH activity were noted in these cells treated with JQ1 alone, while drug combination showed slightly enhanced effect only in the ERG-positive VCaP cells (Fig. 7m–o ). Since ALDHs play a critical role in the maintenance and differentiation of stem cells, we evaluated the efficacy of these two drugs in in vitro using a 3D-prostatosphere assay using VCaP cells. Notably, a significantly decreased number of spheres were formed in cells treated with drug combination than JQ1 alone (Fig. 7p ). Moreover, reduced tumor-sphere forming ability of VCaP cells treated with drug combination group was corroborated by robust decrease in DLX1 expression compared to JQ1 alone (Fig. 7q ). Interestingly, 22RV1 and 42D ENZ R cells failed to show enhanced effect in response to the combinatorial treatment with JQ1 and Enza, signifying the alternative pathways involved in ERG fusion-positive and -negative backgrounds. Collectively, our data reveal the efficacy of JQ1 alone or in combination with Enza for targeting DLX1-driven PCa in an ERG-dependent and -independent manner. BETi abrogates DLX1-mediated tumorigenesis and metastases in mice To investigate the efficacy of BETi against DLX1-mediated tumor growth in vivo, we implanted 22RV1 cells subcutaneously in athymic immunodeficient mice, and when the tumors reached a palpable stage (average volume ~75 mm 3 ); mice were randomized into four groups ( n = 6) and the drugs were administered. We observed that the mice treated with JQ1 alone or a combination of JQ1 and Enza showed almost similar trend in tumor regression (~50% and ~60% at day 19 and 25, respectively) as compared to the vehicle control group, indicating absence of any additive effect with the combinatorial treatment (Fig. 8a, b ). Moreover, no adverse effect on the mice body weight was observed during the course of study (Fig. 8c ). This observation is consistent with our in vitro data, wherein an additive anti-cancer effect with JQ1 and Enza combination was observed in VCaP cells, but not in ERG-negative 22RV1 cells. Furthermore, previous studies have also reported enhanced efficacy of JQ1 and Enza combination than JQ1 alone in VCaP tumors bearing mice [53] . Perhaps, these findings indicate that the additive anti-cancer effect of JQ1 and Enza combination is primarily augmented in ERG -positive background. Next, to determine the impact of drug treatment on spontaneous tumor metastasis, we excised lungs and bone marrow from the mice after terminating the study and isolated genomic DNA, followed by quantitative PCR for detecting human-specific Alu -sequence. We observed a marked decrease in the number of cells metastasized to these organs in both JQ1 alone, or in combination with Enza groups compared to vehicle control (Fig. 8d, e ). Notably, no enhanced effect was observed in the group treated with the drug combination. Subsequently, to investigate the effect of these drugs in the tumor xenografts, we performed IHC staining for cell proliferative marker Ki-67, ALDH1A1, and RNA-ISH for DLX1 expression. As speculated, a significant decrease in the DLX1 expression, accompanied by reduced Ki-67 and ALDH1A1 expression was noted in JQ1 alone as well as in drug combination groups (Fig. 8f, g ). Thus, our in vivo findings establish the therapeutic utility of BETi and anti-androgen in hampering the DLX1-mediated tumorigenesis and metastases. Fig. 8: BET inhibitor alone or in combination with Enzalutamide attenuates DLX1-mediated tumorigenesis and metastases. a Mean tumor volume of xenografts generated by implanting 22RV1 cells in athymic nude mice, and randomized into four treatment groups ( n = 6 each), namely, vehicle control, Enza (20 mg/kg), JQ1 (50 mg/kg), and a combination of Enza and JQ1. b Bar plot showing percent tumor reduction in the treatment groups ( n = 6) compared with the vehicle control group. c Mean body weight of mice ( n = 6 per group) during treated with drugs as mentioned in a . d Scatter dot plot showing number of cells metastasized to the bone in xenografted mice treated with drugs ( n = 6 per group) as mentioned in a . Data represent mean ± SD. e Same as d except cells metastasized to lungs ( n = 6 per group). f Representative images depicting IHC staining for Ki-67, ALDH1A1, and RNA-ISH for DLX1 using formalin-fixed paraffin-embedded tumor xenograft specimens ( n = 5 per group) as a . Scale bar, 50 µm. g Box plots showing quantification of Ki-67, ALDH1A1, and DLX1 expression in the tumor tissue sections ( n = 5) of the mice xenografts as a . Data are presented as box-and-whisker plots indicating median (middle line), 25th and 75th percentile (box), and minimum and maximum values (whiskers). For panels a and b Data represent mean ± SEM. For panels, a two-way ANOVA, Tukey’s multiple comparison test; b two-way ANOVA, Dunnett’s multiple comparison test; d , e , g one-way ANOVA, Tukey’s multiple comparisons test was applied. Source data are provided as a Source Data file. Full size image Taken together, we unraveled ERG- and AR-mediated regulatory mechanisms involved in upregulation of DLX1 in an aggressive subset of PCa patients. We demonstrate that AR along with FOXA1 interacts with ERG as a coregulatory transcription factor, thereby orchestrating DLX1 expression in TMPRSS2-ERG positive background. While, in fusion-negative background, AR and FOXA1 function in an ERG-independent manner, possibly in association with other coregulatory factor(s) to regulate the expression of DLX1 . Thus, this triad of the key regulators control DLX1 expression in a context-dependent manner, resulting in DLX1-mediated oncogenesis via upregulation of several DLX1 target genes and biological processes. Importantly, we also demonstrate pharmacological inhibition of DLX1 transcriptional circuitry by BET inhibitor in an ERG-independent background, and in combination with anti-androgen in an ERG-dependent context (Fig. 9 ). Fig. 9: Schematic showing transcriptional regulation of DLX1 and therapeutic utility of BET inhibitor and anti-androgen in suppressing DLX1-mediated oncogenic effects. Illustration depicting transcriptional regulation of DLX1 via ERG and AR-driven circuitry in ERG fusion-positive background, and through AR/FOXA1 in an ERG-independent context, thereby promoting cancer progression and metastases. In addition, DLX1 drives the expression of its target genes involved in stemness and oncogenesis, such as ALDH1A1 and HNF1A . Utility of BET inhibitor alone or in combination with anti-androgen drugs to target transcriptional regulators of DLX1 resulting in reduced expression of DLX1 and its downstream oncogenesis. Created with BioRender.com. Full size image Molecular biomarker-based diagnostic tests for DLX1 and HOXC6 in post-DRE urine samples have been instrumental in reducing unnecessary biopsies and identifying PCa patients at increased risk of high-grade disease [18] , [54] . Here, we show association of higher DLX1 expression in PCa patients’ specimens with aggressive disease and overall poor survival. Integrative omics approaches such as Tracing Enhancer Networks using Epigenetic Traits (TENET) have identified DLX1 to be associated with over hundred tumor-specific active enhancers in primary PCa patients, thereby implicating the significance of the extensive DLX1 cistrome that contributes to tumor progression [23] . In addition, patient’s positive for both ERG and DLX1 expression exhibit higher Gleason score and poor survival probability, emphasizing the oncogenic cooperativity which may contribute to disease aggressiveness and distant metastases. Similar to ERG-mediated transcriptional regulation of DLX1 , TDRD1 (Tudor Domain Containing 1), another established PCa biomarker has been shown to be differentially regulated in ERG fusion-positive patients, wherein ERG modulates the methylation patterns of the TDRD1 promoter thereby activating its transcription [55] . Furthermore, meta-analysis of gene expression data from five independent PCa studies indicated co-clustering of ERG with DLX1 implicating the hierarchical gene regulatory network of transcription factors [56] , thus suggesting that ERG might modulate the TFs involved in embryonic development. 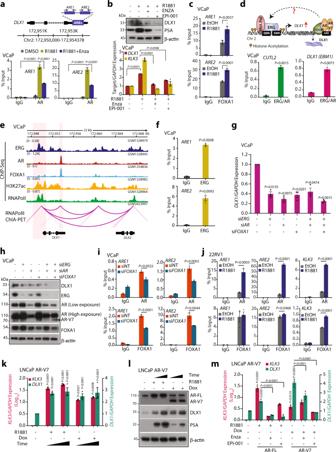Fig. 6: AR and AR-V7 regulate DLX1 expression in both ERG-dependent and -independent manners. aSchematic showing the androgen response elements (AREs) at theDLX1putative enhancer (top panel). ChIP-qPCR data (bottom panel) depicting AR recruitment at theDLX1putative enhancer in R1881 (10 nM) stimulated VCaP cells in the presence or absence of Enzalutamide (Enza, 10 µM) (P< 0.0001).bImmunoblot (top panel) and Q-PCR (bottom panel) data showing relative expression of target genes in VCaP cells under similar culture conditions as indicated.cChIP-qPCR data depicting FOXA1 recruitment at theDLX1putative enhancer in R1881 (10 nM) stimulated VCaP.dSchematic representation showing the possible interaction between ERG and AR on theDLX1promoter (top panel). Re-ChIP data showing co-enrichment of AR and ERG on EBM at theDLX1promoter (bottom panel).eIntegrated genome view of 3D-chromatin structure and binding of transcription factors at the genomic and nearby region ofDLX1.fBar plots depicting ChIP-qPCR data for ERG occupancy at theDLX1enhancer region.gQ-PCR data showing relative expression ofDLX1in siRNA-mediatedERG,AR,and/orFOXA1-silenced VCaP cells.hSame asgexcept immunoblot data.iChIP-qPCR data showing enrichment of AR (top panel) and FOXA1 (bottom panel) in siRNA-mediatedFOXA1-silenced VCaP cells. jChIP-qPCR data depicting AR (top panel) and FOXA1 (bottom panel) enrichment at theDLX1putative enhancer in 22RV1 cells stimulated with R1881 (10 nM) for 16 h.KLK3shown as a positive control.kRelative expression ofKLK3andDLX1in doxycycline (Dox) induced AR-V7 overexpressing LNCaP cells treated with R1881 (10 nM). For induction, 40 ng/ml of Dox or vehicle control was used for 24 and 48 h.lImmunoblots showing the expression of AR-FL, AR-V7, DLX1, and PSA using same cells ask. β-actin used as loading control.mQ-PCR data showingDLX1andKLK3expression in LNCaP AR-V7 cells under similar culture conditions as mentioned at 48-h time point. Data shown from three biologically independent samples (n= 3). Data represent mean ± SEM. For panels,a,bTwo-way ANOVA Sidak’s multiple comparison test;fUnpaired two-tailed Welch’st-test;gOne-way ANOVA, Dunnett’s multiple comparison test;c,i,j,mTwo-way ANOVA, Tukey’s multiple comparisons;kTwo-way ANOVA, Dunnett’s multiple comparison test was applied. Source data are provided as a Source Data file. In corroboration with these independent studies, our findings draw attention to the hierarchical regulatory network between ERG and DLX1, wherein the emergence of TMPRSS2-ERG fusion as an early event in primary PCa results in direct transcriptional upregulation of DLX1 via ERG/AR contributing to disease progression. Collateral to this, we discovered an association between DLX1 and AR expression irrespective of TMPRSS2-ERG fusion status, and the role of AR signaling in transcriptional regulation of DLX1 in ERG-independent context. Progression of CRPC is supported by sustained AR signaling which is predominantly dependent on the expression of constitutively active ligand-independent AR-V7 [9] . Several studies reported AR transcriptional cistrome reprogramming in metastatic CRPC, wherein a cellular context-dependent transcriptional network operates downstream of AR which is distinct from the AR transcriptional program engaged in androgen-dependent stage [57] . Furthermore, genome-wide AR binding profiles [57] demonstrated a highly complex transcriptional circuitry, where AR possibly functions through enhancers distant from the promoters to impart regulation of target genes [2] , [3] . Although it has been shown that ERG represses AR expression and inhibits AR-mediated transcriptional regulation of canonical genes [3] , several reports show the cooperativity between these TFs, where AR binds at the enhancer region and forms chromatin loop to interact with ERG at gene promoters thereby regulating the expression of downstream target genes [5] , [49] . Recent advancements in understanding the genomic interactions and chromatin looping using high throughput sequencing and conformation capture techniques provided important insight into the high-resolution 3D-chromatin landscape of normal and PCa cells [50] . Moreover, the crucial information about the mapping of RNA-Pol II, AR, and ERG in PCa demonstrates the long- and short-range interactions of these TFs orchestrating genomic expression in PCa [49] , [50] . In line with these studies, our data suggest the formation of an active transcriptional complex involving recruitment of AR-FL along with FOXA1 at the putative enhancer region of DLX1 , which also interacts with ERG occupied DLX1 promoter in fusion-positive cases, and possibly with other coregulatory TFs in the fusion-negative context. We speculate that this short-range chromatin loop structure between the enhancer-promoter region of DLX1 is further enabled by the RNA-Pol II-associated interaction at DLX1 genomic region, implicating the AR-driven transcriptional activation of DLX1 in an ERG-dependent and -independent manner. Besides, our results also indicate the enrichment of AR-V7 at the putative enhancer region of DLX1 and further reveal the role of constitutively activated AR-signaling in regulating its expression. Conclusively, these findings demonstrate the role of AR signaling wherein both AR-FL and AR-V7 regulate DLX1 transcriptional activation in advanced stage PCa. It is known that AR facilitates transcriptional regulation by partnering with transcriptional co-regulators such as histone deacetylases (HDACs), bromodomain-containing proteins (BRDs) as well as ETS TFs such as ERG [12] , [49] , [58] . Moreover, BETi are shown to attenuate AR and ERG-mediated oncogenesis in CRPC by disrupting transcriptional activation complex at their target gene loci [2] , [12] , [59] . Currently, therapeutic targeting of bromodomain proteins has gained clinical importance for the treatment of several malignancies including CRPC, for instance, BETi such as OTX-015, ZEN003694, and GS-5829 are already in clinical trials as single agents or in combination with anti-androgens for CRPC patients [60] . Alongside, our results demonstrate the potency of BETi alone and in combination with anti-androgen to reduce the expression of DLX1 and its target genes, thus, implicating the utility of DLX1 as a therapeutic target. Concomitantly, we also suggest that the enhanced effectiveness of drug combination (BETi and anti-androgen) is plausibly predominant in ERG fusion-positive background. Our findings show that BETi along with anti-androgens could be used to mitigate the oncogenic effects of DLX1 via disrupting AR and ERG transcriptional circuitries and can be considered as a potential therapeutic intervention in the treatment of the ERG+/DLX1+ subtype of PCa. Although, TMPRSS2-ERG gene fusion is the highly prevalent genetic alteration in PCa, unlike gene fusions involving oncogenic kinases (e.g., RAF-kinase fusions) [61] , transcription factors such as ERG are challenging to target. Recent advancements with the development of small molecular inhibitors, peptidomimetics [62] , and proteolysis-targeting chimera (PROTAC) [63] show promise in targeting transcription factors in cancers, thus paving a way to exploit DLX1 as a potential drug target. Taken together, this study moved the field forward by providing strong evidence to employ parallel treatment regimens with BETi or/and AR targeted therapeutics for the clinical management of DLX1-positive PCa subtype, hence opening new treatment avenues for patients with advanced-stage disease. In silico data processing and computational analysis To study the association of DLX1 with PCa, The Cancer Genome Atlas – Prostate Adenocarcinoma (TCGA-PRAD) dataset was downloaded from UCSC Xena browser ( https://xenabrowser.net ) and analyzed for DLX1 gene expression. The samples were sorted according to the tissue type and data was plotted for DLX1 expression (log 2 (norm_count+1)) in solid normal tissue ( n = 52) against primary PCa tissue ( n = 498) using GraphPad prism version 7.0. No cut-off was applied on the dataset. Similar analysis was applied on the data retrieved from Gene Expression Omnibus (GEO) database with accession number GSE35988. For GSE80609, similar analysis was applied for TCGA-PRAD except FPKM values were plotted. For Kaplan–Meier survival analysis, survival data of patients with primary tumors were considered. Days to first biochemical recurrence and up to last follow-up for TCGA-PRAD patients were the parameters taken into account for the analysis. Samples were divided into two groups based on the expression level of DLX1 using Cox proportional hazards regression model in R version 3.6.1. 5-year survival probability was calculated using Kaplan–Meier survival analysis by applying survival package ( https://cran.r-project.org/web/packages/survival ), and log-rank test was used to detect statistical significance. For survival analysis of patients with varying DLX1 expression and its association with other TCGA-defined PCa subtypes (including ERG), data was obtained from UALCAN database [37] . For the heatmap representation, hierarchical clustering was performed on expression data using heatmap.2 function of gplot package in R version 3.6.1. No cut-off was applied on the TCGA dataset for correlation plot of ERG and DLX1 . Correlation plot between ERG and DLX1 in TCGA-PRAD and MSKCC dataset was directly retrieved from GEPIA [64] and cBioPortal [65] , respectively. SU2C data downloaded from cBioPortal was classified into two groups based on the ERG -fusion status, and the Pearson correlation graph was plotted using GraphPad prism. To identify putative target genes of DLX1, publicly available ChIP-Seq data for DLX1 in LoVo colorectal cancer cell lines were analyzed, and the genes with enrichment of DLX1 were shortlisted and were overlapped with genes downregulated in microarray expression data of 22RV1- DLX1 -KO cells. Common genes present at the intersection were considered as DLX1 putative target genes. Bioinformatics analysis of sequencing data We analyzed the publicly available RNA-Seq data using Galaxy [66] , a web platform available on the public server at https://usegalaxy.org . Raw sequencing FASTQ reads were prefetched and Fastq-dumped using SRA-toolkit ( http://ncbi.github.io/sra-tools/ ). Followed by this, reads were assessed for their quality using FASTQC, followed by trimming of data using Trimmomatic. The adapter trimmed reads were next aligned to the human reference genome (hg19) using HISAT2 to obtain binary alignment map (BAM) files. Read alignment results were visualized using Integrative Genomic Browser (IGB) [67] in reference to the human genome. Next, the transcript abundance among different conditions was analyzed using FeatureCounts. Differential gene expression profiles were evaluated using DESeq2 to produce a list of differentially expressed genes with log 2 fold change (FC) and FDR corrected P -values. Genes were annotated using the Entrez gene IDs and those with adjusted P -value < 0.05 were selected. Next, differential expressed genes were sorted such that genes with log 2 FC > 0 were considered upregulated while those with log 2 FC < 0 were considered downregulated. Pathway enrichment analysis was performed by using DAVID [68] and GSEA [69] . Volcano plot was generated using Galaxy online server. ChIP-sequencing data analysis of online available datasets on GEO was performed. Galaxy web platform was used to perform ChIP-Seq analysis with default settings. Raw single-end reads in FASTQ format were uploaded to the web server using the NCBI SRA accession number for individual samples followed by FASTQC and sequence trimming with FASTQ Trimmer. Next, Sequence Alignment Map (SAM) files were generated by read alignment to the reference human genome (version as mentioned in the respective study) using Bowtie. Aligned reads were further filtered for the unmapped reads and were converted to the Binary Alignment Maps (BAM) file using SAMtools. ChIP-Seq peak calling was done using Model-based analysis of ChIP-Seq (MACS; P < 10 −5 ) data with default settings against respective controls. MACS output files were visualized using IGB. RNA-Pol II ChIA-PET data (GSM3423997) was downloaded from GEO and visualized using integrated genome viewer (IGV) [70] . Cell lines culture conditions and authentication Prostate cancer cell lines (22RV1, VCaP, LNCaP, PC3) and benign prostate epithelial cells (RWPE1) were obtained from the American Type Culture Collection (ATCC) and were cultured as per the ATCC recommended guidelines. Using specific culture medium was supplemented with 10% fetal bovine serum (FBS) and 0.5% Penicillin-Streptomycin (Gibco Thermo-Fisher), cells were cultured in incubator supplied with 5% CO 2 at 37 °C (Thermo Scientific). Enzalutamide-resistant 42D ENZ R cells were obtained as a kind gift from Dr. Amina Zoubeidi [71] . For authenticating the cell line identity, short tandem repeat (STR) profiling was performed at the Lifecode Technologies Private Limited, Bangalore, and DNA Forensics Laboratory, New Delhi. Mycoplasma contamination test was routinely carried out for all the cell lines using PlasmoTest mycoplasma detection kit (InvivoGen). Establishing DLX1 knockout cell line CRISPR/Cas9 knockout (KO) kit was purchased from Origene (KN206895) and KO cell lines were generated following the manufacturer’s protocol. 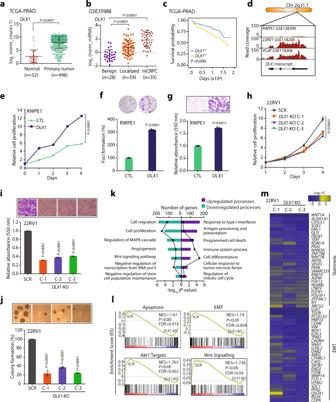Briefly, pCas-guide vector containing guide RNA (gRNA) sequence (specific to DLX1 and scramble control) along with donor vector containing homologous arms and functional cassette were co-transfected in the host 22RV1 cells. Cells were passaged up to eight generations post-transfection to eliminate the extrachromosomal donor vector and were then grown under puromycin (Sigma-Aldrich) selection (1 µg/ml) pressure to select the positive clones. Single-cell colonies were picked and cultured followed by screening at the genomic level. PCR was performed using the primers spanning the deleted genomic region in DLX1 gene. The DLX1-KO cells were further validated for loss of DLX1 at the transcript and protein levels using qPCR and immunoblot, respectively (described elsewhere). Fig. 1: High DLX1 expression associates with poor prostate cancer prognosis and promotes disease progression. aDot plot showingDLX1expression in PCa patients (n= 498) and matched normal (n= 52) in TCGA-PRAD RNA-Seq dataset, data represents log2 (norm_count+1), center depicts mean ± (standard deviation) SD (P< 0.0001).bDot plot ofDLX1expression using microarray profiling data (GSE35988) comprising benign (n= 28), localized (n= 59), and mCRPC (n= 35) patient specimens, data represents log2 (norm_mRNA), center depicts mean ± SD (P< 0.0001).cKaplan–Meier plot showing survival probability in TCGA-PRAD (n= 498) dataset categorized in highDLX1(DLX1Hi) and lowDLX1(DLX1Lo) expression.dRNA-Seq data showingDLX1transcript read counts in publicly available datasets (GSE128399 and GSE118206).eCell proliferation assay using isogenic RWPE1 cells overexpressing DLX1 at indicated time-points (P< 0.0001).fFoci formation assay using same cells ase(P< 0.0001).gBoyden Chamber Matrigel migration assay using same cells ase(P< 0.0001). Representative images for panelsf(scale bar 500 µm) andg(scale bar 100 µm) are shown as inset.hCell proliferation assay using 22RV1-DLX1-KO (C-1, C-2, and C-3 are independent clones) and control cells at indicated time-points (P< 0.0001).iBoyden Chamber Matrigel migration assay using same cells ash(P< 0.0001).jAnchorage-independent soft agar assay using same cells ash(P< 0.0001). Representative images for panelsiandjare shown as inset (scale bar 100 µm).kDAVID analysis showing upregulated (right) and downregulated (left) biological processes in 22RV1-DLX1-KO against control cells. Bars represent the −log10(P-value) and the frequency polygon (black line) denotes number of genes.lSame ask, except gene set enrichment analysis (GSEA) plots representing deregulated pathways.mHeatmap displaying downregulated genes involved in cancer stemness and EMT in 22RV1-DLX1-KO cells compared to control. Data shown from three biologically independent samples (n= 3). Data represent mean ± SEM unless specified. For panels,aUnpaired Student’s two-tailedt-test was applied;bOne-way ANOVA with Dunnett’s multiple comparison test was applied;eTwo-way ANOVA Sidak’s multiple comparison test;f,gUnpaired two-tailed Welch’st-test;hTwo-way ANOVA, Dunnett’s multiple comparisons test;i,jOne-way ANOVA, Dunnett’s multiple comparisons test was applied. Source data are provided as a Source Data file. Primer sequences are provided in Supplementary Table 1 . Plasmids and constructs Briefly, DLX1 cDNA was cloned in pCDH lentiviral vector (Addgene) to establish DLX1 overexpressing cell lines. The pHAGE AR-V7 and control vectors were obtained as a kind gift from Dr. Nancy Weigel [72] . Successful lentiviral packaging of these constructs was performed to generate stable cell lines (described elsewhere). pGL3-Basic vector, a kind gift from Dr. Amitabha Bandyopadhyay at IIT Kanpur, was used to perform promoter reporter assay. For luciferase reporter assays, ~1 kb promoter region of DLX1 was cloned in pGL3-Basic vector and site-directed mutagenesis was performed to mutate the ERG binding motifs (EBMs) in the DLX1 promoter. Primer sequences used for mutagenesis are provided in Supplementary Table 1 . Lentiviral packaging Lentiviral particles for pCDH vectors were generated using third-generation ViraPower Lentiviral Packaging Mix (Invitrogen) according to the manufacturer’s protocol. For pHAGE vectors, second-generation pMD.2G and psPAX2 packaging systems were procured from Dr. Subba Rao Gangi Setty at the Indian Institute of Science, Bangalore. Briefly, packaging mix was co-transfected with lentiviral vector in HEK293FT cells using FuGENE HD Transfection Reagent (Promega). Media containing transfection reagent was replenished with complete growth media after 24 h. The lentiviral particles were harvested after 48–60 h, were aliquoted, and stored in −80 °C freezer. For establishing stable cell lines, host cells were transduced with viral particles in a 6-well dish along with Polybrene (hexadimethrine bromide; 8 µg/ml) (Sigma-Aldrich) to increase the transduction efficiency. Media was replaced 24 h later, followed by selection of transduced cells under appropriate antibiotic pressure. To generate DLX1 overexpressing RWPE1 cells, pCDH-DLX1 vector was used for infection, and cells were selected in puromycin (0.5 µg/ml). LNCaP AR-V7 cells were selected under Geneticin (Gibco, ThermoFisher Scientific) at a concentration of 350 µg/ml. RWPE1-ERG overexpression and control cells were cultured in Keratinocyte SFM Media (ThermoFisher) along with supplements provided by the manufacturer. siRNA transfection VCaP cells plated at confluency of 40-45% in a six-well dish were transfected with 30 pmol of siRNA against DLX1 , ERG , AR , FOXA1 , and non-targeting control (Dharmacon). Lipofectamine RNAiMAX transfection reagent (ThermoFisher Scientific) was used according to the manufacturer’s protocol. After 24 h, cells were transfected again, and 36 h post second transfection, they were harvested for functional assays. Likewise, transient DLX1 knockdown was performed in 42D ENZ R cells. For ChIP-qPCR in VCaP, cells were plated in a 100 mm dish followed by transfection using siRNA against FOXA1 . Functional assays For cell proliferation assay, about 1 × 10 4 cells per well were seeded in a 12-well culture dish, and cells were counted using hemocytometer at the indicated time points. Alternatively, Resazurin (Cayman Chemicals) was added to the cells (2 × 10 3 ) plated in 96-well dish and fluorescence was measured with emission-excitation at 590–530 nm. The relative cell proliferation rate was plotted against the indicated time points. Foci formation assay was performed by plating ~2 × 10 3 cells in a six-well culture dish containing the recommended growth media in reduced serum (5% FBS) condition. Cells were incubated at 37 °C for three weeks by replacing media every third day. Paraformaldehyde (4% in 1× PBS) was used to fix the cells followed by staining with crystal violet solution (0.05% w/v), and number of foci were counted for quantification. Cell migration assay was performed using 8 μm pore size of Transwell Boyden chamber (Corning). Growth media supplemented with 20% FBS was added to the lower compartment, followed by seeding 1 × 10 5 cells suspended in serum-free culture media to the Transwell inserts. Cells were incubated at 37 °C, 24 h later migrated cells were fixed in paraformaldehyde (4% in 1× PBS) and stained using crystal violet (0.5% w/v). 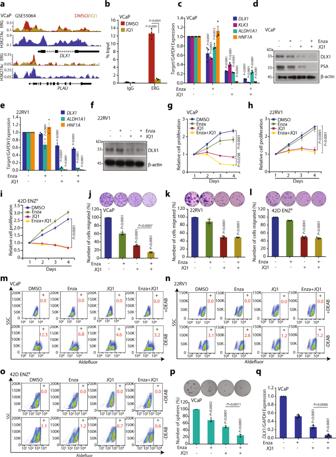Fig. 7: BET inhibitor alone or in combination with Enzalutamide downregulates DLX1 expression and mitigates its oncogenic properties. aChIP-Seq data (GSE55064) showing ERG enrichment onDLX1promoter in VCaP cells treated with JQ1 or vehicle control for 24 h. H3K27Ac represents active promoter in untreated cells.PLAUused as a positive control.bChIP-qPCR data showing relative ERG enrichment onDLX1promoter in VCaP cells treated with JQ1 (0.5 µM) for 48 h (P< 0.0001).cQ-PCR data showing relative expression of target genes in VCaP cells treated with Enza (10 µM), JQ1 (0.5 µM) alone or in combination for 48 h.KLK3used as a positive control for JQ1 treatment.dSame ascexcept immunoblot. β-actin was used as loading control.eSame ascexcept 22RV1 cells.fSame aseexcept immunoblot (P< 0.0001).gCell proliferation assay in VCaP cells treated with drug conditions as mentioned inc.hSame asgexcept 22RV1 cells (P< 0.0001).iSame asgexcept 42D ENZRcells (P< 0.0001).jBoyden Chamber Matrigel migration assay in VCaP cells using same treatment conditions asc. Inset shows representative image of the migrated cells (scale bar 30 µm).kSame asjexcept 22RV1 cells (scale bar 30 µm,P< 0.0001).lSame asjexcept Enza-resistant, 42D ENZRcells (scale bar 30 µm,P< 0.0001).mFluorescence intensity of the catalyzed ALDH substrate in VCaP cells under same treatment conditions asc. Marked windows show ALDH1+ percent cell population.nSame asmexcept 22RV1 cells.oSame asmexcept 42D ENZRcells.pBar plot showing number of spheres formed in prostatosphere assay using VCaP under same treatment conditions asc. Inset shows representative image of the spheres formed (scale bar 100 µm).qQ-PCR data for theDLX1expression using RNA isolated from VCaP prostatospheres. Data shown from three biologically independent samples (n= 3). Data represent mean ± SEM. For panelsb,c,etwo-way ANOVA, Tukey’s multiple comparison test;g,h,iOne-way ANOVA, Dunnett’s multiple comparison test;j–l,p,qOne-way ANOVA, Tukey’s multiple comparison was applied. Source data are provided as a Source Data file. Cells adhered onto Transwell filter were de-stained in 10% v/v acetic acid followed of quantification at absorbance at 550 nm. Migrated cells were visualized and captured using upright Nikon microscope. For cells treated with drug, number of migrated cells stained with crystal violet were counted using ImageJ software. For anchorage-independent soft agar assay, 0.6% low melting-point agarose (Sigma-Aldrich) dissolved in RPMI-1640 medium was poured in six-well culture dishes. After polymerization, another layer of 0.3% soft agar in RPMI-1640 medium containing cells (~1.5 × 10 4 ) was poured on the top of the first layer. Cells were incubated for 20 days at 37 °C, and colonies >40 μm in size were counted. Real-time quantitative PCR To identify relative target gene expression, total RNA extracted using TRIzol (Ambion) was converted into cDNA using First Strand cDNA synthesis kit (Genetix Biotech Asia Pvt. Ltd) according to the manufacturer’s instructions. Quantitative PCR (qPCR) was performed on the StepOne Real-Time PCR System (Applied Biosystems) using cDNA template, specific primer sets, and SYBR Green PCR Master-Mix (Genetix Biotech Asia Pvt. Ltd). Primer sequences are provided in Supplementary Table 1 . Immunoblotting Whole-cell protein lysates were prepared in radioimmunoprecipitation assay buffer (RIPA buffer) supplemented with Phosphatase Inhibitor Cocktail Set-II (Calbiochem) and protease inhibitor (VWR), and protein sample was quantified by BCA assay, followed by protein separation on SDS-PAGE. Proteins were then transferred on the PVDF membrane (GE Healthcare), and the membrane was blocked with 5% non-fat dry milk in tris-buffered saline, 0.1% Tween 20 (TBS-T) for 1 h at room temperature. PVDF membrane was incubated overnight at 4 °C with the following primary antibodies at 1:1000 dilution: DLX1 (Thermo, PA5-28899), E-Cadherin (CST, 3195), Vimentin (Abcam, ab92547), phospho-Akt (CST, 13038), total-Akt (CST, 9272), Caspase-3 (CST, 9662), Cleaved PARP (CST, 9541), Bcl-xL (CST, 2764), ERG (Abcam, ab92513), FOXA1 (CST, 58613), 1:2000 diluted AR (CST, 5153), 1:2000 diluted PSA (CST, 5877), and 1:5000 diluted β-actin (Abcam, ab6276). Subsequently, PVDF membranes were washed with 0.1% 1× TBS-T followed by incubation at room temperature for 2 h with secondary anti-mouse or anti-rabbit antibody conjugated with horseradish peroxidase (HRP) (1:5000, Jackson ImmunoResearch Laboratories, Cat # 115-035-003 and Cat # 111-035-144, respectively). Membranes were again washed with 1× TBS-T buffer, and the signals were visualized by enhanced chemiluminescence system (Thermo) according to the manufacturer’s instructions. Gene expression analysis Global gene expression profiling and identification of differentially regulated genes were performed as previously described [73] . 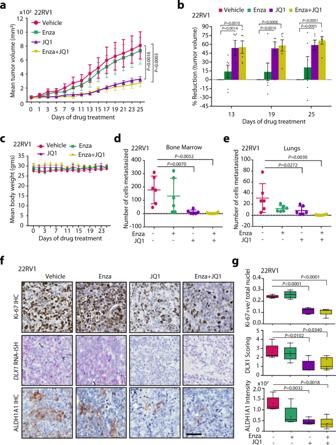Fig. 8: BET inhibitor alone or in combination with Enzalutamide attenuates DLX1-mediated tumorigenesis and metastases. aMean tumor volume of xenografts generated by implanting 22RV1 cells in athymic nude mice, and randomized into four treatment groups (n= 6 each), namely, vehicle control, Enza (20 mg/kg), JQ1 (50 mg/kg), and a combination of Enza and JQ1.bBar plot showing percent tumor reduction in the treatment groups (n= 6) compared with the vehicle control group.cMean body weight of mice (n= 6 per group) during treated with drugs as mentioned ina.dScatter dot plot showing number of cells metastasized to the bone in xenografted mice treated with drugs (n= 6 per group) as mentioned ina. Data represent mean ± SD.eSame asdexcept cells metastasized to lungs (n= 6 per group).fRepresentative images depicting IHC staining for Ki-67, ALDH1A1, and RNA-ISH forDLX1using formalin-fixed paraffin-embedded tumor xenograft specimens (n= 5 per group) asa. Scale bar, 50 µm.gBox plots showing quantification of Ki-67, ALDH1A1, andDLX1expression in the tumor tissue sections (n= 5) of the mice xenografts asa. Data are presented as box-and-whisker plots indicating median (middle line), 25th and 75th percentile (box), and minimum and maximum values (whiskers). For panelsaandbData represent mean ± SEM. For panels,atwo-way ANOVA, Tukey’s multiple comparison test;btwo-way ANOVA, Dunnett’s multiple comparison test;d,e,gone-way ANOVA, Tukey’s multiple comparisons test was applied. Source data are provided as a Source Data file. 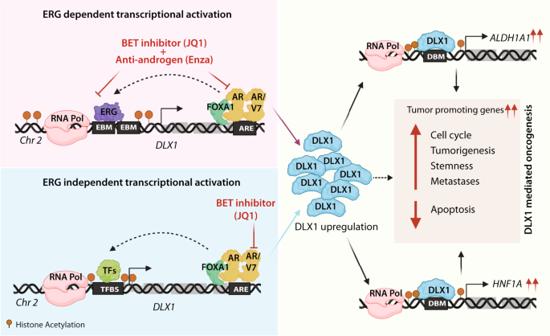Fig. 9: Schematic showing transcriptional regulation ofDLX1and therapeutic utility of BET inhibitor and anti-androgen in suppressing DLX1-mediated oncogenic effects. Illustration depicting transcriptional regulation ofDLX1via ERG and AR-driven circuitry inERGfusion-positive background, and through AR/FOXA1 in an ERG-independent context, thereby promoting cancer progression and metastases. In addition, DLX1 drives the expression of its target genes involved in stemness and oncogenesis, such asALDH1A1andHNF1A. Utility of BET inhibitor alone or in combination with anti-androgen drugs to target transcriptional regulators ofDLX1resulting in reduced expression of DLX1 and its downstream oncogenesis. Created with BioRender.com. Briefly, total RNA from 22RV1- DLX1 -KO and 22RV1-SCR control cells was isolated and subjected to Agilent Whole Human Genome Oligo Microarray profiling (dual color) according to manufacturer’s protocol using Agilent platform (8 × 60 K format). Differentially regulated genes were filtered to only include significantly altered genes with ~1.6-fold average change (log 2 FC >0.6 or <−0.6, P < 0.05). DAVID bioinformatics platform ( https://david.ncifcrf.gov ) was used to identify deregulated biological processes. GSEA was employed to detect gene enrichment in different datasets. Network-based analysis of biological pathways was generated using Enrichment Map, a plug-in for Cytoscape network visualization software [74] ( http://baderlab.org/Software/EnrichmentMap/ ). Flow cytometry For cell cycle distribution, cells were trypsinized and fixed in 70% ethanol followed by staining with propidium iodide (PI) (BioLegend, Cat # 421301) using manufacture’s protocol. Cell cycle distribution was analyzed using in-built univariate model of FlowJo software. For apoptotic studies, cells were dissociated using StemPro™ Accutase™ (ThermoFisher Scientific) and were washed with cold 1× PBS and resuspended in 1× binding buffer (1 × 10 6 cells/ml). Subsequently, 1 × 10 5 cells were stained using PE Annexin V Apoptosis Detection Kit I (BD Biosciences, Cat # 559763) following to the manufacture’s protocol. Quadrants were gated on Annexin (PE) versus 7AAD (PerCP) channel dot plots using unstained, Annexin V (PE), and 7AAD (PerCP) single stained cells as controls. The quadrants were defined as lower left quadrant Annexin − /7AAD − (viable), Annexin + /7AAD − lower right quadrant (early apoptotic), Annexin − /7AAD + upper left quadrant (necrotic), Annexin + 7AAD + upper right quadrant (late apoptotic) cells. Data were acquired on the Beckman Coulter’s CytoFLEX platform and BD FACSMelody™ Cell Sorter and was analyzed using FlowJo software v10.6.1. Aldefluor assay was performed to determine aldehyde dehydrogenase (ALDH) enzymatic activity using Aldefluor kit (Stem Cell Technologies, Catalog #01700) following manufacturer’s guidelines. Briefly, cells were trypsinized and washed with 1× PBS followed by resuspension in 1 ml of Aldefluor assay buffer. Activated Aldefluor substrate (5 μL) was added to the cells and were divided in two conditions, with and without ALDH inhibitor, diethylaminobenzaldehyde (DEAB). After 30 min of incubation at 37 °C, cells were centrifuged and resuspended in 500 μL of Aldefluor assay buffer. The ALDH activity was detected in FITC channel. Gate was applied to identify viable-cell population using forward scatter (FSC) and side scatter (SSC) dot plot. Next, dot plot was generated with FITC channel versus SSC and gate on the control population was applied using DEAB treated samples. The same gate was applied over corresponding samples without DEAB to identify ALDH-positive population. For data acquisition, Beckman Coulter’s CytoFLEX platform and BD FACSMelody™ Cell Sorter were used. The analysis was performed using FlowJo software v10.6.1. For stem cell markers, cells were stained with PE/Cy7 anti-human CD44 antibody (Miltenyi Biotec, 130-113-904, 1:50) and CD338-PE (ABCG2-PE, Miltenyi Biotec, 130-105-010, 1:40) followed by 1-h incubation at 4 °C. Firstly, gate was applied to identify viable-cell population using FSC and SSC dot plot. Histograms were generated for antibody-stained samples and were compared to their isotype controls. Data acquisition was carried out by using Beckman Coulter’s CytoFLEX platform and BD FACSMelody™ Cell Sorter. Data were analyzed with FlowJo software v10.6.1. Gating strategies applied for the flow cytometry experiments are provided in Supplementary Fig. 7 . Mice xenograft study NOD.CB17- Prkdc scid /J (NOD/SCID) (Jackson Laboratory), five to six-week-old male mice were anesthetized using ketamine and xylazine (50 mg/kg and 5 mg/kg, respectively) cocktail injected intraperitoneally. 22RV1- DLX1 -KO and 22RV1-SCR control cells were trypsinized and were suspended (2 × 10 6 ) in 100 μl of saline with 20% Matrigel and implanted subcutaneously at the dorsal both flank sides of mice ( n = 6 for each condition). Tumor burden was measured using digital Vernier caliper on alternate days, and tumor volume was calculated using formula (π/6) ( L × W 2 ), ( L = length; W = width). To examine spontaneous metastases from the xenograft study, lungs and bone marrow of the xenografted mice were excised at the end of the study and analyzed by performing Taqman assay using primers specific for human Alu -sequences as mentioned in Supplementary Table 1 . Briefly, genomic DNA was isolated from the harvested organs and TaqMan probe FAM-YB8-ALU-167 (Applied Biosystems) with sequence 5′-6-FAM-AGCTACTCGGGAGGCTGAGGCAGGA-TAMRA-3′ (position 167–192) was used [31] , which specifically hybridize to the human-specific YB8-Alu sequence. For generating standard curve Taqman assay was performed by using serially diluted human gDNA spiked with mouse gDNA, and accordingly based on the CT values number of metastasized cells were determined [31] . For experimental metastases experiment, athymic nude (NU(NCr)- Foxn1 nu ), 5–6-week-old male mice procured from Hylasco Biotechnology Pvt. Ltd. (distributor for Charles River Research Models) were anesthetized. 22RV1-SCR or DLX1 -KO cells (4 × 10 5 ) were resuspended in 20 µl of saline and implanted by intramedullary tibial injections using 26-gauge needle. Piroxicam (3 mg/kg) was administered intramuscular post-implantation to reduce the pain. After 4 weeks, mice were subjected to X-ray scan and were euthanized. Tibia subjected to injections were harvested and analyzed using micro-CT. To investigate the anti-tumorigenic effect of BETi and anti-androgen in mice xenograft model, 5–6-week-old male athymic nude (NU(NCr)- Foxn1 nu ) mice were subcutaneously implanted with 22RV1 (3 × 10 6 ) cells at both sides of dorsal flank. Mice were randomized into four groups ( n = 6 per group) once the average tumor volume reached 75 mm 3 and treated with vehicle control, enzalutamide (20 mg/kg), JQ1 (50 mg/kg) or JQ1 and Enza combination for 5 days a week. Enza diluted in 5% dimethyl sulfoxide (DMSO), 30% polyethylene glycol 400 (PEG-400) (Sigma-Aldrich), 65% corn oil (Sigma-Aldrich) was administered by oral gavage, while JQ1 diluted in 10% cyclodextrin (Sigma-Aldrich) was administered intraperitonially for 4 weeks. Tumor burden and mice weight was measured every alternate day. At the end of the experiment, mice were sacrificed after 4 h of drug treatment. Tumor, bone marrow, and lungs were excised for further characterization. Spontaneous metastasis to lungs and bone marrow was examined using TaqMan assay as described earlier. All immunodeficient mice used in the study were housed in specific-pathogen-free (SPF) facility as per the guidelines. The ambient temperature of the mice facility room was maintained at 20–24 °C with ~40–60% humidity and 12:12 h light–dark cycle. Micro-computed tomography (microCT) The analysis of the bone lesions and bone morphometric parameters was performed using microCT (Bruker microCT SKYSCAN). The scanning parameters used for performing microCT include resolution of 7 and 0.5 µm Al filter. Medium pixel setting with 48 kV and 204 µA of current with rotation step at 0.6 was used. The total time elapsed to scan each sample was 29 min. 3D image reconstruction and visualization were performed using volume rendering program CTVox. The CTAn v1.16.8.0 software was used for 3D image processing and parametric analysis. IHC of tumor xenografts and patients’ specimens Tumor tissues excised from xenografted mice were fixed in 10% buffered formalin, followed by paraffin embedding and sectioning at 3 µm thickness using microtome (Leica). After deparaffinization and rehydration of tissue sections, heat-induced antigen-retrieval was performed using sodium citrate buffer (pH 6.0). Next, endogenous peroxidase activity was quenched using 3% hydrogen peroxide (H 2 O 2 ) for 10 min, followed by blocking tissue sections in 5% normal goat serum, and were incubated with primary antibodies against Ki-67 (CST, 9449 S), E-Cadherin (CST, 3195), and Vimentin (Abcam, ab92547) at 4 °C overnight. After washing with tris-buffered Saline (TBS), sections were incubated with biotinylated secondary antibody at room temperature for 1 h followed by incubation with ABC (Avidin-Biotin complex) (Vector Labs) for 30 min. Sections were then processed for detection of HRP activity using DAB (3, 3-diaminobenzidine) peroxidase (HRP) substrate kit (Vector Labs). Quantification for Ki-67 using 15 random histological fields was performed using ImageJS Ki-67 online module [75] and proliferation rate was calculated by normalizing Ki-67 positive nuclei with respect to total nuclei. For quantification of E-cadherin, Vimentin, and ALDH1A1 integrated density was calculated using IHC Toolbox in ImageJ software using 15 random histological fields. Alternatively, PCa patient specimens and tumor xenograft slides were incubated at 60 °C for 2 h followed by target retrieval in a PT Link instrument (Agilent DAKO, PT200) using EnVision FLEX Target Retrieval Solution, High pH (Agilent DAKO, K800421-2). 1X EnVision FLEX Wash Buffer (Agilent DAKO, K800721-2) was used to wash slides followed by treatment with Peroxidazed 1 (Biocare Medical, PX968M) and Background Punisher (Biocare Medical, BP974L) for 5 min wash after each step. Slides were incubated with ERG [EPR3864] (Abcam, ab92513), AR (CST, 5153), Ki-67 (Agilent, IR626), and ALDH1A1 (CST, 54135) antibodies overnight at 4 °C. Afterward, slides were washed and then incubated in Mach2 Doublestain 1 (Biocare Medical, MRCT523L) for 30 min at room temperature, and then rinsed in 1X EnVision wash buffer and treated with a Ferangi Blue solution (Biocare Medical, FB813S). Next, slides were rinsed in distilled water followed by treatment with EnVision FLEX Hematoxylin (Agilent DAKO, K800821-2). After rinsing in tap water, slides were dried completely and then dehydrated using xylene. EcoMount (Biocare Medical, EM897L) was added to each slide, which was then mounted with coverslips. RNA in situ hybridization (RNA-ISH) For RNA-ISH, slides incubated at 60 °C were de-paraffinized in xylene. Slides were then kept in 100% ethanol twice for 3 min each and then air-dried following treatment with H 2 O 2 for 10 minutes. Further, slides were rinsed and boiled in 1X Target Retrieval for 15 min. After rinsing slides in distilled water, Protease Plus treatment was given and then incubated with DLX1 probe (Advanced Cell Diagnostics, probe ID: 569601) for 2 h at 40 °C. Next, slides were washed and treated with Amp 1 for 30 minutes, Amp 2 for 15 min, Amp 3 for 30 min, and Amp 4 for 15 min, all steps were carried out at 40 °C in the HybEZ oven with two washes in 1× Wash Buffer. Slides were then treated with Amp 5 for 30 min and Amp 6 for 15 min at room temperature in a humidity chamber. Red color was developed by adding a 1:60 solution of Fast Red B: Fast Red A to each slide and incubating for 10 min. Finally, slides were treated with EnVision FLEX Hematoxylin (Agilent DAKO, K800821-2) and mounted using the same protocol as used for IHC slides. ERG and DLX1 staining evaluation ERG IHC staining was evaluated to define ERG positive and negative status of PCa tissues. DLX1 expression was identified by scoring the signal intensity of RNA-ISH probe hybridization for the TMA foci and the number of red dots/cell were evaluated to grade DLX1 expression into four levels ranging from score of 0–3 as described previously [76] . Next, an association between the expression of ERG and DLX1 was calculated by applying Chi-Square contingency test on GraphPad Prism version 7.0. Chromatin immunoprecipitation (ChIP) All ChIP experiments were performed as described previously [77] . Briefly, crosslinked cells were lysed using lysis buffer [1% SDS, 10 mM EDTA, 50 mM Tris-Cl, and protease inhibitor (Genetix)] followed by sonication for DNA fragmentation to an average fragment length of ~500 bp using Bioruptor (Diagenode). Sheared chromatin was incubated at 4 °C overnight with 4 µg of primary or isotype control antibodies. Antibodies against ERG (abcam, ab92513), H3K9Ac (CST, 9649), Rpb1 CTD/RNA PolII (CST, 2629), AR (CST, 5153), DLX1 (Thermo, PA5-28899), control rabbit IgG (Invitrogen, 10500C) and control mouse IgG (Invitrogen, 10400C) were used to perform ChIP assays. Simultaneously, the Protein G coated Dynabeads (Invitrogen) were blocked with BSA (HiMedia) and sheared salmon sperm DNA (Sigma-Aldrich), followed by incubation at 4 °C overnight. Blocked beads were incubated for 6–8 h at 4 °C with the lysate containing antibody to make antibody-bead conjugates. Next, the beads conjugated with antibody were washed and immunocomplex was eluted using elution buffer [1% SDS, 100 mM NaHCO 3 , Proteinase K (Sigma-Aldrich) and RNase A (500 µg/ml each) (Sigma-Aldrich)]. DNA was isolated using phenol-chloroform-isoamyl alcohol extraction method. Binding sites for ERG transcription factor in the DLX1 promoter were identified using JASPAR and MatInspector software. For Re-ChIP, first ChIP was performed using ERG antibody eluted in 10 mM DTT in Tris-EDTA buffer at 37 °C for 30 min, subsequently, DTT-elute was further diluted 50 times and second round of ChIP was performed following the similar protocol using antibody against AR. The ChIP-qPCR was performed using primers provided in Supplementary Table 1 . Luciferase reporter assay Isogenic RWPE1-CTL and RWPE1-ERG cells plated in 24-well culture dish, and were transfected with pGL3-DLX1-P wildtype (250 ng) and pRL-null vector (2.5 ng) using FuGENE HD Transfection Reagent. After 48 h of incubation at 37 °C, cells were harvested using the lysis buffer provided with Dual-Glo Luciferase assay kit (Promega). GloMax® 96 Microplate Luminometer (Promega) was used to measure the Firefly and Renilla luciferase activity according to the manufacturer’s protocol. Renilla luciferase activity was used as a normalization control. The same protocol was followed to measure the luciferase promoter reporter activity for pGL3-DLX1-P mutant construct. Androgen stimulation and drug treatment For androgen stimulation, cells were serum-starved for 72 h in phenol-red free media supplemented with 5% charcoal-stripped serum (CSS) (Gibco), followed by stimulation with 10 nM R1881 (Sigma-Aldrich) at the indicated time points. For anti-androgen treatment, VCaP cells were cultured in phenol-red free DMEM media supplemented with GlutaMAX (Gibco) and 5% CSS followed by pre-treatment with anti-androgen for 6 h. Next, cells were stimulated with 1 nM R1881 in the presence of anti-androgen for 48 h. The same procedure was followed for anti-androgen treatment in LNCaP cells, except RPMI-1640 phenol-red free medium (Gibco) was used. For ChIP-qPCR experiments, VCaP and 22RV1 cells were stimulated with 10 nM R1881 for 16 h. For VCaP anti-androgen ChIP experiment, cells were pre-treated with Enzalutamide for 6 h followed by stimulation with R1881 in the presence of anti-androgen for 16 h. For BETi and anti-androgen treatment, cells were grown in complete growth media followed by JQ1 and Enza treatment at 0.5 µM and 10 µM concentrations, respectively. The same concentration was used for combinatorial treatment. For functional assays and flow cytometry, cells were plated in six-well dish and treated with JQ1 and Enza at the above-mentioned concentrations for 48 h and were processed for further characterization. Prostatosphere assay VCaP cells (2 × 10 4 ) were plated in low adherence 6-well dish and were cultured in serum-free DMEM-F12 media (1:1, Invitrogen) supplemented with B27 (1X, Invitrogen), EGF (20 ng/ml, Invitrogen), and FGF (20 ng/ml, Invitrogen). Cells were allowed to grow and the spheroids formed were collected and mechanically dissociated to form a single-cell suspension before replating them in fresh media. The cells were then treated with DMSO, Enza, and/or JQ1 by adding them in the fresh media. Cells were passaged regularly and drugs were replenished in fresh media at each passage. Experiment was terminated after three weeks and the prostatospheres formed in all the groups were counted and imaged. At the end of the study, spheroids were harvested for isolating RNA as described earlier. Statistics For statistical analysis, one-way ANOVA, two-way ANOVA, unpaired two-tailed Student’s t- test, and Unpaired two-tailed Welch’s t -test was used for independent samples or otherwise mentioned in the respective figure legend. For P -value <0.05, the differences between the groups were considered significant. Significance was indicated as follows: * P < 0.05, ** P < 0.005, and *** P < 0.001. Error bars represent the standard error of the mean (SEM) obtained from experiments performed at least three independent times. Study approval All mice experiment procedures were approved by the Committee for the Purpose of Control and Supervision of Experiments on Animals (CPCSEA) and abide to all regulatory standards of the Institutional Animal Ethics Committee of the Indian Institute of Technology Kanpur. TMAs comprising prostate cancer specimens ( n = 144) were obtained from the Department of Pathology, Henry Ford Health System (Detroit, MI). These patients were not administered with any hormone therapy, except for three. Metastatic CRPC patients TMA was obtained from the Department of Urology, University of Washington, Seattle. Biospecimens were obtained within 8 h of death from patients who died of metastatic CRPC. Visceral metastases were identified at the gross level, bone biopsies were obtained from 16 to 20 different sites and metastases identified at a histological level. Tissues were fixed in buffered formalin (bone metastases were decalcified in 10% formic acid) and embedded in paraffin and were used to construct the TMA using duplicate 1 mm diameter cores from these tissues. Institutional Review Board approvals from the Henry Ford Health System (IRB#10375) and University of Washington (IRB#2341) and informed consents were received from the participants prior to inclusion in the study. All patients’ specimens used in this study were collected in accordance with the Declaration of Helsinki. Reporting summary Further information on research design is available in the Nature Research Reporting Summary linked to this article.